Synaptic recruitment of gephyrin regulates surface GABAAreceptor dynamics for the expression of inhibitory LTP Postsynaptic long-term potentiation of inhibition (iLTP) can rely on increased GABA A receptors (GABA A Rs) at synapses by promoted exocytosis. However, the molecular mechanisms that enhance the clustering of postsynaptic GABA A Rs during iLTP remain obscure. Here we demonstrate that during chemically induced iLTP (chem-iLTP), GABA A Rs are immobilized and confined at synapses, as revealed by single-particle tracking of individual GABA A Rs in cultured hippocampal neurons. Chem-iLTP expression requires synaptic recruitment of the scaffold protein gephyrin from extrasynaptic areas, which in turn is promoted by CaMKII-dependent phosphorylation of GABA A R-β3-Ser 383 . Impairment of gephyrin assembly prevents chem-iLTP and, in parallel, blocks the accumulation and immobilization of GABA A Rs at synapses. Importantly, an increase of gephyrin and GABA A R similar to those observed during chem-iLTP in cultures were found in the rat visual cortex following an experience-dependent plasticity protocol that potentiates inhibitory transmission in vivo . Thus, phospho-GABA A R-β3-dependent accumulation of gephyrin at synapses and receptor immobilization are crucial for iLTP expression and are likely to modulate network excitability. Inhibition in the central nervous system is involved in many processes, including dendritic computation, network oscillations and selection of cell assemblies [1] . Changes in inhibitory synaptic strength are thus expected to profoundly affect network function. Over the last decade, accumulating evidence has shown that inhibitory synapses exhibit several forms of long-term plasticity, expressed at either the presynaptic or postsynaptic level [2] . Although inhibitory plasticity at the presynaptic level has been extensively characterized [2] , the detailed mechanisms of postsynaptic inhibitory plasticity remain elusive. Postsynaptic forms of long-term potentiation of inhibition (iLTP) have been shown to involve (i) changes in channel function [3] , [4] ; (ii) changes in GABA A receptor (GABA A R) intracellular trafficking [5] , [6] ; or (iii) alterations in the intracellular chloride concentration [7] . Interestingly, some of these types of synaptic plasticity depend on the activation of Ca 2+ /calmodulin-dependent kinase II (CaMKII) [3] , [6] , [8] , [9] . A key role of CaMKII has been shown in the cerebellum, when low-frequency stimulation of climbing fibres potentiates GABAergic synapses formed by stellate/basket cells onto cerebellar Purkinje neurons [8] . Likewise, in hippocampal cultured neurons and slices, moderate activation of N -methyl- D -aspartate receptor (NMDAR) causes selective translocation of activated CaMKII to inhibitory synapses [10] and CaMKII-dependent exocytosis of GABA A Rs, leading to a persistent enhancement of GABAergic synaptic currents [5] . Importantly, despite the clear demonstration that enhanced receptor intracellular trafficking is involved in postsynaptic iLTP expression, the fine mechanisms that regulate GABA A R clustering and stabilization at synapses during potentiation of inhibition are not fully elucidated. Surface neurotransmitter receptors, including AMPARs (α-amino-3-hydroxy-5-methyl-4-isoxazolepropionic acid receptors), mGluRs (metabotropic glutamate receptors), NMDARs, GlyRs and GABA A Rs, have been reported to laterally diffuse between synaptic and extrasynaptic compartments, contributing to the regulation of receptor number at synapses under basal conditions [11] , [12] and during synaptic plasticity [13] , [14] , [15] , [16] , [17] . The impact of receptor lateral diffusion on synaptic plasticity has been extensively studied at excitatory synapses, where LTP-inducing stimuli lead to the rapid immobilization of synaptic AMPARs [14] , [17] . In contrast, the regulation of GABA A R lateral diffusion during plasticity at inhibitory synapses is poorly understood. Recently, it has been reported that iLTD increases the mobility of GABA A Rs, leading to receptor dispersal from inhibitory synapses [13] , [15] , [16] , whereas GABA A R surface dynamics during iLTP has never been investigated. Synaptic clustering and surface lateral mobility of neurotransmitter receptors are largely modulated by the interaction between receptors and intracellular scaffold proteins [11] . This has been directly demonstrated for AMPAR–PSD95–stargazin, mGluR–Homer and GlyR–gephyrin interactions [12] . At GABAergic synapses, gephyrin is involved in the clustering of GABA A Rs [6] , [18] , [19] , [20] . In keeping with this, the direct binding between gephyrin and several subunits of GABA A R (α1–3 and β2–3) has been reported [21] , [22] , [23] , [24] . However, GABA A R clustering at synapses can also occur in a gephyrin-independent manner, at least for some GABA A R subunits [23] , [25] , [26] , [27] , thus indicating that other proteins of the inhibitory postsynaptic scaffold can participate in GABA A R stabilization at synapses [26] , [27] , [28] , [29] . Notably, in basal conditions, gephyrin can influence the lateral mobility of GABA A Rs at synapses as demonstrated by depletion and lateral dispersion of synaptic GABA A Rs on gephyrin impairment [19] . In contrast, the involvement of gephyrin in iLTP expression has never been addressed. Here we investigate the mechanisms of postsynaptic iLTP at the single protein level. We demonstrate for the first time that iLTP expression depends on gephyrin recruitment at synapses, promoted by CaMKII-dependent phosphorylation of the GABA A R β3 S383 residue. As a consequence of gephyrin recruitment, GABA A Rs are immobilized at synapses as demonstrated by single-particle tracking (SPT) of GABA A Rs labelled with Quantum Dots (QDs). We also show that increased perisomatic accumulation of gephyrin and GABA A Rs is observed in principal cells of the rodent visual cortex after monocular deprivation, a manipulation of the rat visual input that is known to elicit iLTP in vivo [30] , [31] , [32] . Together, these results demonstrate the causal link between receptor phosphorylation and GABA A R/gephyrin synaptic accumulation during iLTP. CaMKII mediates synaptic GABA A R immobilization during iLTP To induce postsynaptic potentiation of GABAergic synapses in cultured hippocampal neurons (16–18 days in vitro (DIV), see Methods), we adopted a chemical protocol based on moderate NMDAR activation [5] (NMDA 20 μM, 6-cyano-7-nitroquinoxaline-2,3-dione (CNQX) 10 μM for 2 min). This protocol ( Fig. 1a , upper panel) caused a persistent 41±7% ( n =18; P <0.001, one-way analysis of variance (ANOVA), followed by Dunnett’s post test, Fig. 1a,b ) increase in the amplitude of miniature GABAergic synaptic currents (mIPSCs) and, similarly, the potentiation of the amplitude of spontaneous inhibitory postsynaptic currents (sIPSCs) ( Supplementary Fig. 1a,b ) and of evoked GABAergic currents ( Supplementary Fig. 1c,d ). Importantly, these forms of NMDA-induced potentiation of inhibition lasted up to 30 min, thus allowing referring to as chemically induced iLTP (chem-iLTP) ( Supplementary Fig. 1a–e ). The molecular modifications occurring during chem-iLTP were analysed 20 min after stimulation, when potentiation reached the steady state. The NMDA-mediated potentiation of mIPSCs amplitude was prevented by 10 min treatment with the CaMKII inhibitor KN-62 (3 μM) and by adding BAPTA (1,2-bis( o -aminophenoxy)ethane- N,N,N′,N′ -tetraacetic acid, 11 mM) in the recording pipette to avoid an increase of intracellular Ca 2+ ( P <0.001, one-way ANOVA, followed by Dunnett’s post test, Fig. 1a,b ), thus suggesting a postsynaptic mechanism. In line with this, after NMDA stimulation, the total number of GABA A Rs and their postsynaptic accumulation were increased in a CaMKII-dependent manner, as revealed by immunolabelling for surface GABA A R α1 subunit. Indeed, NMDA-treated neurons exhibited an increase in total surface GABA A Rs average immunoreactivity that was prevented by KN-62 (sham: 40.4±1.4 a.u. per pixel, n =23; NMDA: 48.4±2.5 a.u. per pixel, n =24; NMDA/KN-62: 39.7±1.6 a.u. per pixel, n =24, one-way ANOVA, followed by Newman–Keuls’ post test). Similarly, NMDA-induced enhancement of the density and intensity of synaptic GABA A Rs clusters was blocked by KN-62 treatment (clusters per 100 μm: sham=65.2±10.2 a.u., n =23; NMDA=122.5±16.1 a.u., n =24; NMDA/KN-62=90.5±13.1 a.u., n =24; one-way ANOVA, followed by Newman–Keuls’ post test. GABA A R integrated fluorescence intensity: Sham=1,701±93 a.u. ; NMDA=2,200±154 a.u. ; NMDA/KN-62=1,449±92 a.u. ; n =24 in each condition; one-way ANOVA, followed by Newman–Keuls’ post test) ( Fig. 1c,d ). Importantly, these results were accompanied by an unaffected density of vGAT-positive puncta after NMDA application ( Supplementary Fig. 1g ), thus arguing against changes in the number of GABAergic synapses during chem-iLTP. To further investigate the postsynaptic features of the NMDA-induced potentiation of synaptic current amplitude, we next aimed at dissecting out the possibility that chem-iLTP was due to an actual increase of receptor number or to changes in receptor single-channel conductance. The non-stationary fluctuation analysis performed on evoked IPSCs (eIPSCs) recorded before and 20 min after the stimulation showed that after NMDA treatment GABA A Rs single-channel conductance was not altered, whereas the number of open receptors at the current peak significantly increased ( Supplementary Fig. 1h ). Taken together, these data demonstrate that NMDA-dependent iLTP is expressed at the postsynaptic level through an increased number of synaptic receptors and depends on CaMKII-mediated activity. 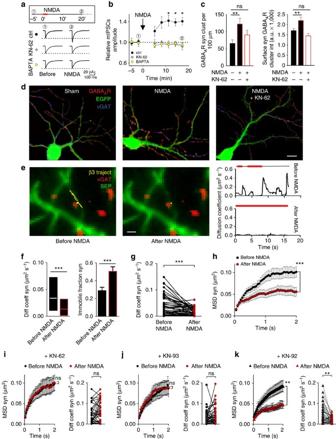Figure 1: GABAAreceptors are immobilized at GABAergic synapses during chem-iLTP. (a) Top: outline of the protocol applied to induce chem-iLTP. The red bar indicates NMDA application. ‘1’ and ‘2’ represent the time points for quantifications before and 20 min after NMDA stimulation; lower panel: representative averaged mIPSCs traces before (‘1’) and after (‘2’) NMDA treatment, in control (ctrl), CaMKII blockade (KN-62) and intracellular Ca2+buffering (BAPTA (1,2-bis(o-aminophenoxy)ethane-N,N,N',N'-tetraacetic acid)). (b) Time course of mIPSCs amplitude increase after NMDA application (arrow) in control (n=18) and KN-62 (n=12) or BAPTA (n=12). (c) Effect of NMDA on GABAAR (α1-subunit) synaptic cluster density (left) and integrated fluorescence intensity (right) with or without KN-62. (d) Representative confocal images of GABAAR (α1-subunit, red) and vGAT (blue) immunoreactivity in EGFP-expressing neurons (green) after sham (left) or NMDA treatment, with (middle) or without (right) KN-62. Scale bar, 10 μm. (e) Left: representative trajectories (yellow) of an individual β3-containing GABAAR diffusing on a SEP-β3-transfected neuron (green) live stained for presynaptic vGAT (red) before and after NMDA application. Scale bar, 1 μm. SeeSupplementary Movie 1. Right: diffusion coefficient versus time plot of the QD-labelled receptor on the left, before and after NMDA. Lines above curves represent QD synaptic (red) and extrasynaptic (black) localization. (f) Median diffusion coefficient and IQR (left) of all synaptic GABAARs (ntrajectories=365) before and after NMDA (ntrajectories=351, 26 neurons;P<0.001, Mann–WhitneyU-test) and the corresponding immobile fraction (right) (P<0.001, Student’st-test). (g) Matched diffusion coefficients of individual GABAARs at synapses before (black) and after NMDA treatment (red) (ntrajectories=67 out of 351–365 reported inf,P<0.001, paired Wilcoxon test). (h) MSD versus time values of matched observations of individual GABAARs before and after NMDA (ntrajectories=67 from 26 neurons,P<0.001, pairedt-test). (i–k) Quantifications of matched observations of synaptic GABAARs before and after NMDA in the presence of the indicated drugs.ntrajectories: (i) KN-62=38 from 16 neurons, (j) KN-93=53 from 19 neurons; (k) KN-92=ntrajectories=51 from 18 neurons. Top: diffusion coefficients, paired Wilcoxon test; bottom: MSD versus time plot, pairedt-test at steady state. Unless otherwise stated, error bars represent s.e.m. *P<0.05; **P<0.01; ***P<0.005; ns, nonsignificant. Figure 1: GABA A receptors are immobilized at GABAergic synapses during chem-iLTP. ( a ) Top: outline of the protocol applied to induce chem-iLTP. The red bar indicates NMDA application. ‘1’ and ‘2’ represent the time points for quantifications before and 20 min after NMDA stimulation; lower panel: representative averaged mIPSCs traces before (‘1’) and after (‘2’) NMDA treatment, in control (ctrl), CaMKII blockade (KN-62) and intracellular Ca 2+ buffering (BAPTA (1,2-bis( o -aminophenoxy)ethane- N,N,N',N' -tetraacetic acid)). ( b ) Time course of mIPSCs amplitude increase after NMDA application (arrow) in control ( n =18) and KN-62 ( n =12) or BAPTA ( n =12). ( c ) Effect of NMDA on GABA A R (α1-subunit) synaptic cluster density (left) and integrated fluorescence intensity (right) with or without KN-62. ( d ) Representative confocal images of GABA A R (α1-subunit, red) and vGAT (blue) immunoreactivity in EGFP-expressing neurons (green) after sham (left) or NMDA treatment, with (middle) or without (right) KN-62. Scale bar, 10 μm. ( e ) Left: representative trajectories (yellow) of an individual β3-containing GABA A R diffusing on a SEP-β3-transfected neuron (green) live stained for presynaptic vGAT (red) before and after NMDA application. Scale bar, 1 μm. See Supplementary Movie 1 . Right: diffusion coefficient versus time plot of the QD-labelled receptor on the left, before and after NMDA. Lines above curves represent QD synaptic (red) and extrasynaptic (black) localization. ( f ) Median diffusion coefficient and IQR (left) of all synaptic GABA A Rs ( n trajectories =365) before and after NMDA ( n trajectories =351, 26 neurons; P <0.001, Mann–Whitney U -test) and the corresponding immobile fraction (right) ( P <0.001, Student’s t -test). ( g ) Matched diffusion coefficients of individual GABA A Rs at synapses before (black) and after NMDA treatment (red) ( n trajectories =67 out of 351–365 reported in f , P <0.001, paired Wilcoxon test). ( h ) MSD versus time values of matched observations of individual GABA A Rs before and after NMDA ( n trajectories =67 from 26 neurons, P <0.001, paired t -test). ( i – k ) Quantifications of matched observations of synaptic GABA A Rs before and after NMDA in the presence of the indicated drugs. n trajectories : ( i ) KN-62=38 from 16 neurons, ( j ) KN-93=53 from 19 neurons; ( k ) KN-92= n trajectories =51 from 18 neurons. Top: diffusion coefficients, paired Wilcoxon test; bottom: MSD versus time plot, paired t -test at steady state. Unless otherwise stated, error bars represent s.e.m. * P <0.05; ** P <0.01; *** P <0.005; ns, nonsignificant. Full size image To understand whether the lateral diffusion of GABA A Rs contributes to changes in receptor number at inhibitory synapses during chem-iLTP, the mobility of individual QD-coupled GABA A Rs was monitored by SPT before and after NMDA stimulation (see Methods). These experiments describe the mobility of receptors present at the neuronal surface at the beginning of the experiment, as QD labelling was performed before the stimulation. The effects of NMDA treatment on the lateral mobility of GABA A Rs was first probed on cultured hippocampal neurons (DIV 16–18) transfected with GABA A R β3 subunit at DIV 7. NMDA stimulation strongly immobilized recombinant β3-GABA A Rs at synapses ( Fig. 1e ) by reducing the diffusion coefficient of mobile receptors (median diffusion coefficient and interquartile range (IQR) before=0.034 μm 2 s −1 , IQR: 0.012–0.073, n trajectories =365; after=0.013 μm 2 s −1 , IQR: 0.002–0.032; P <0.001, Mann–Whitney U -test) and by promoting a massive increase in the fraction of immobile receptors (before: 0.29±0.04; after NMDA: 0.50±0.05; P <0.001, Student’s t -test) ( n trajectories : before=365, after=351 from 26 neurons; Fig. 1f and Supplementary Movie 1 ). This result was reinforced by matched observations of the same GABA A Rs present at synapses before and 20 min after stimulation, showing that receptor diffusion coefficients were significantly reduced after NMDA application ( n =67 trajectories out of 351–365, P <0.001, paired Wilcoxon test, Fig. 1g ). Those effects were paralleled by increased GABA A R confinement at synapses as indicated by the reduced steady state of the mean square displacement (MSD) curve ( P <0.001, paired t -test at steady state, Fig. 1h ). In sham-treated controls, the diffusive properties of synaptic and extrasynaptic GABA A Rs remained stable over the duration of the experiment ( Supplementary Fig. 2a,b ). It is worth mentioning that NMDA stimulation did not alter the lateral mobility of extrasynaptic GABA A Rs ( Supplementary Fig. 2c ), suggesting that the immobilization observed during chem-iLTP was selective for synaptic receptors. To assess the reliability of our SPT data on recombinant β3 subunits, the lateral mobility of endogenous α1 subunits was studied during chem-iLTP. The diffusion properties of native synaptic and extrasynaptic α1-containing GABA A Rs before and after NMDA stimulation were indistinguishable from those of transfected β3-containing GABA A Rs ( Supplementary Fig. 2d–g ). Given the CaMKII dependence of chem-iLTP, we next examined the role of CaMKII in the immobilization of synaptic GABA A R during potentiation of inhibition. On treatment with KN-62 (3 μM), the mobility of all synaptic GABA A R was not affected by NMDA stimulation ( n trajectories =202–211 from 16 neurons; P >0.05, Mann–Whitney U -test; Supplementary Fig. 2h ). Consistently, matched observations of synaptic GABA A Rs before and after NMDA application revealed unchanged diffusion coefficient and confinement at synapses in the presence of KN-62 ( n trajectories =38 out of 202–211; P >0.05, paired Wilcoxon test, Fig. 1i ). As a control, we observed that under basal conditions, KN-62 treatment did not affect the mobility of synaptic GABA A R ( Supplementary Fig. 2i ). Similar to KN-62, KN-93 (5 μM), an alternative inhibitor of CaMKII activity, prevented the NMDA-induced immobilization and confinement of GABA A Rs at synapses, leaving receptor lateral diffusion at synapses unaffected by NMDA ( n trajectories =258–265 from 19 neurons; Supplementary Fig. 2j ; matched observations n trajectories =53 out of 258–265, Fig. 1j ). On the contrary, on treatment with KN-92 (5 μM), an inactive analogue of KN-93, the lateral mobility of synaptic GABA A R was significantly reduced and confined after NMDA stimulation ( n trajectories =216–222 from 18 neurons, Supplementary Fig. 2k ; matched observations n trajectories =51 out of 216–222, Fig. 1k ). The possibility that internalization of QD-receptor complexes during the experiment duration might affect the measurements of QD-receptor lateral mobility was assessed with the acid strip procedure to remove surface antibodies (see Methods). The lack of residual QDs when the acid strip was performed 25 min after QD labelling confirms that over this time span the SPT approach exclusively monitors surface receptors due to minimal QD receptor internalization ( Supplementary Fig. 3 ). Altogether, these data indicate that during chem-iLTP, pre-existing surface GABA A Rs are immobilized at synapses via a CaMKII-dependent mechanism. Catalytic activity of CaMKII is required for iLTP To confirm that the catalytic activity of CaMKII is involved in NMDA-mediated iLTP, we overexpressed a CaMKII-K42R mutant, known to impair CaMKII-mediated phosphorylation [33] . NMDA treatment failed to significantly potentiate mIPSCs amplitude in neurons transfected (at DIV 7) with CaMKII-K42R-mCherry (9.7±8.7%, n =12) as compared with neurons transfected with the control plasmid mCherry (43.3±10.9%, n =12; one-way ANOVA, followed by Dunnett’s post test, Fig. 2a,b ). Next, the mobility of synaptic GABA A Rs on impairment of CaMKII kinase activity was studied after chem-iLTP induction with SPT experiments. In agreement with the electrophysiology results, the diffusion coefficients and the immobile fraction of β3-containing GABA A Rs in neurons expressing CaMKII-K42R-mCherry were not affected by the stimulation protocol and exhibited comparable values before and after NMDA treatment ( n trajectories : before=246; after=231 from 15 neurons; Fig. 2c ). On the contrary, β3-containing GABA A Rs tracked in control neurons expressing mCherry confirmed a significant reduction of the median diffusion coefficient and an increase in the immobile fraction after NMDA application ( n trajectories : before=198; after=184, from 14 neurons; Fig. 2c ). Along the same lines, matched observations of GABA A R-QD complexes before and 20 min after NMDA treatment demonstrated that CaMKII-K42R overexpression prevents the NMDA-induced drop of synaptic receptor mobility and the increased receptor confinement at synapses observed in control neurons (matched observations n trajectories :control=36 out of 184–198; CaMKII-K42R=50 out of 231–246; Fig. 2d,e ). 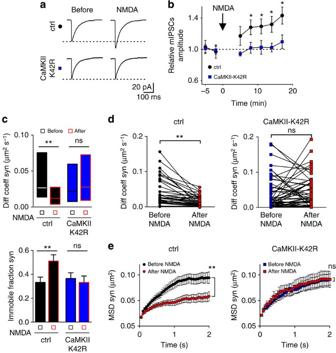Figure 2: GABAAreceptor immobilization at GABAergic synapses during chem-iLTP depends on CaMKII kinase activity. (a) Example averaged traces of mIPSCs recorded before and after NMDA application from neurons overexpressing CaMKII-K42R-mCherry or mCherry alone as a control. (b) Quantification over time of the relative increase of mIPSCs amplitude after stimulation in control (mCherry) and in CaMKII-K42R-mCherry-expressing neurons (n=12 in each condition). (c) Median diffusion coefficient (top, one-way ANOVA, followed by Dunn’s post test) and immobile fraction (bottom, one-way ANOVA, followed by Bonferroni post test) of synaptic GABAARs tracked in neurons overexpressing the kinase dead mutant CaMKII-K42R (n=231–246 from 15 neurons) or in control cultured hippocampal cells (n=184–198 from 14 neurons). (d) Matched diffusion coefficients of individual synaptic GABAARs before (black) and after NMDA treatment (red) in control neurons (ntrajectories=36 out of 184–198,P<0.01, paired Wilcoxon test) and on overexpression of CaMKII-K42R. (ntrajectories=50 out of 231–246,P<0.05, paired Wilcoxon test). (e) MSD over time plot of matched individual GABAARs observed at synapses before and after NMDA in control (ntrajectories=36,P=0.008, pairedt-test) and in CaMKII-expressing neurons (ntrajectories=50,P>0.05, pairedt-test). Error bars represent s.e.m. *P>0.05; **,P<0.01 and ns, nonsignificant. Figure 2: GABA A receptor immobilization at GABAergic synapses during chem-iLTP depends on CaMKII kinase activity. ( a ) Example averaged traces of mIPSCs recorded before and after NMDA application from neurons overexpressing CaMKII-K42R-mCherry or mCherry alone as a control. ( b ) Quantification over time of the relative increase of mIPSCs amplitude after stimulation in control (mCherry) and in CaMKII-K42R-mCherry-expressing neurons ( n =12 in each condition). ( c ) Median diffusion coefficient (top, one-way ANOVA, followed by Dunn’s post test) and immobile fraction (bottom, one-way ANOVA, followed by Bonferroni post test) of synaptic GABA A Rs tracked in neurons overexpressing the kinase dead mutant CaMKII-K42R ( n =231–246 from 15 neurons) or in control cultured hippocampal cells ( n =184–198 from 14 neurons). ( d ) Matched diffusion coefficients of individual synaptic GABA A Rs before (black) and after NMDA treatment (red) in control neurons ( n trajectories =36 out of 184–198, P <0.01, paired Wilcoxon test) and on overexpression of CaMKII-K42R. ( n trajectories =50 out of 231–246, P <0.05, paired Wilcoxon test). ( e ) MSD over time plot of matched individual GABA A Rs observed at synapses before and after NMDA in control ( n trajectories =36, P =0.008, paired t -test) and in CaMKII-expressing neurons ( n trajectories =50, P >0.05, paired t -test). Error bars represent s.e.m. * P >0.05; **, P <0.01 and ns, nonsignificant. Full size image In the attempt to additionally provide a more holistic description of the mobility of all surface GABA A Rs during synaptic potentiation at inhibitory synapses and the contribution of CaMKII activity in this process, fluorescence recovery after photobleaching (FRAP) experiments were performed in control neurons and neurons exhibiting impaired CaMKII activity due to CaMKII-K42R overexpression at DIV 7. The mobility of GABA A Rs was estimated from the recovery of super-ecliptic-pHluorin (SEP)-tagged-β3 fluorescence in photobleached synaptic areas visualized by live vGAT staining (see Methods) before and after NMDA stimulation on the same neuron. The pH sensitivity of SEP-β3 ( Supplementary Fig. 4a–d ) demonstrates that these FRAP experiments describe the mobility of only surface receptors. After NMDA treatment in control mCherry-expressing neurons, SEP-β3 fluorescence recovery at synapses was significantly reduced as compared with basal conditions (before: 45±2 %, n =56; after NMDA: 38±2 %, n =69; Supplementary Fig. 4e,f , Student’s t -test), suggesting a global lower GABA A R mobility at synapses on plasticity induction. This effect was prevented by the overexpression of the inactive CaMKII, as the fluorescence recovery of SEP-β3 was comparable before (45±2%, n =61) and after NMDA treatment in CaMKII-K42R-mCherry-transfected neurons (44±3%, n =70 synapses from seven neurons in three neuronal preparations; Supplementary Fig. 4e,f ). Overall, these experiments show that CaMKII activity is required for the immobilization of surface GABA A Rs at inhibitory synapses during synaptic potentiation of inhibition. Phosphorylation of GABA A R-β3 Ser 383 is essential for iLTP In another set of experiments we examined whether CaMKII phosphorylation of GABA A Rs could contribute to chem-iLTP expression. Among the potential phosphorylation sites identified on GABA A R subunits, only the Ser 383 residue of the β3 subunit is exclusively phosphorylated by CaMKII [34] with direct functional implications on GABA A R-mediated currents [35] , [36] . The possible involvement of Ser 383 phosphorylation by CaMKII in chem-iLTP expression was directly tested with a specific anti-phospho-β3Ser 383 antibody [36] in immunoblot assays before and at various time points (10 and 20 min) after the stimulation protocol ( Fig. 3a ). Although the levels of Ser 383 phosphorylation remained constant at all time points in sham-treated hippocampal cultures, in NMDA-treated neurons the phosphorylation of β3Ser 383 progressively increased, becoming significant 20 min after stimulation ( n =8; P =0.04, one-way ANOVA followed by Dunn’s post test; Fig. 3b ). 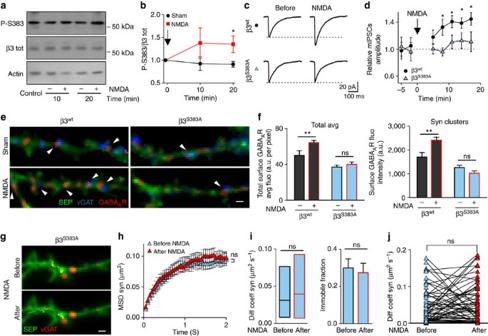Figure 3: Phosphorylated S383 of GABAAR β3 subunit allows iLTP through GABAAR accumulation and immobilization at synapses. (a) Representative immunoblots of phosphoS383 and total β3 detected in non-treated control neurons and in neurons treated with NMDA or with a sham solution (arrow) and subsequently allowed different recovery periods as indicated. Actin immunoreactivity (lower panel) is to check equal loading. (b) Quantification of phosphoS383/total β3 band intensity ratio normalized to control (n=8 in each condition,P=0.04, one-way ANOVA followed by Dunn’s post test). (c) Representative averaged mIPSC recordings from the same β3wt- or β3S383A-expressing neuron before and after NMDA. (d) Lack of relative mIPSCs amplitude increase after NMDA application (arrow) on overexpression of β3S383A(cyan,P>0.05) as compared with β3wt(black,P=0.03) (in each condition:n=10, one-way ANOVA followed by Dunnett’s post test). (e) Representative confocal images of neurons expressing SEP-β3wt(left, green) or SEP-β3S383A(right, green) immunostained for GABAAR (α1-subunit, red), vGAT (blue) treated with sham solution or NMDA. Arrowheads indicate GABAAR synaptic clusters. Scale bar, 5 μm. (f) NMDA-induced increase of total surface GABAAR average immunoreactivity and GABAAR synaptic cluster integrated fluorescence intensity observed in β3wt-expressing neurons (black) are prevented by the S383A mutation on β3 subunit (cyan) (total β3wt: sham=50±5 a.u. per pixel, NMDA=65±2 a.u. per pixel; total β3S383A: sham=37±2 a.u. per pixel; NMDA=40±2 a.u. per pixel;n=24 in each condition, one-way ANOVA, followed by Newman–Keuls’ post test) (synaptic cluster intensity β3wt: sham=1,700±190 a.u., NMDA=2,401±131 a.u.; β3S383A: sham=1,258±100 a.u.; NMDA=1,023±96 a.u.;n=24 in each condition, one-way ANOVA, followed by Newman–Keuls’ post test). (g) Comparable trajectories (yellow) of an individual SEP-β3S383A-containing GABAAR coupled to a QD before and after NMDA treatment. vGAT is represented in red. Scale bar, 1 μm. See alsoSupplementary Movie 2. (h) Matched MSD over time plot of individual β3S383Areceptors observed at synapses before and after NMDA (ntrajectories=61, 17 neurons,P>0.05, pairedt-test). (i) Synaptic β3S383Areceptors before and after NMDA treatment exhibit comparable median diffusion coefficient (and IQR) (ntrajectories: before=272; NMDA=263, 17 neurons;P>0.05, Mann–WhitneyU-test) and immobile fraction (P>0.05, Student’st-test). (j) Matched diffusion coefficients of individual β3S383Areceptors present at synapses before and after NMDA (ntrajectories=61 out of 236–272;P>0.05, paired Wilcoxon test). Unless otherwise stated, error bars represent s.e.m. *P<0.05; **P<0.01; ns, nonsignificant. Figure 3: Phosphorylated S383 of GABA A R β3 subunit allows iLTP through GABA A R accumulation and immobilization at synapses. ( a ) Representative immunoblots of phosphoS383 and total β3 detected in non-treated control neurons and in neurons treated with NMDA or with a sham solution (arrow) and subsequently allowed different recovery periods as indicated. Actin immunoreactivity (lower panel) is to check equal loading. ( b ) Quantification of phosphoS383/total β3 band intensity ratio normalized to control ( n =8 in each condition, P =0.04, one-way ANOVA followed by Dunn’s post test). ( c ) Representative averaged mIPSC recordings from the same β3 wt - or β3 S383A -expressing neuron before and after NMDA. ( d ) Lack of relative mIPSCs amplitude increase after NMDA application (arrow) on overexpression of β3 S383A (cyan, P >0.05) as compared with β3 wt (black, P =0.03) (in each condition: n =10, one-way ANOVA followed by Dunnett’s post test). ( e ) Representative confocal images of neurons expressing SEP-β3 wt (left, green) or SEP-β3 S383A (right, green) immunostained for GABA A R (α1-subunit, red), vGAT (blue) treated with sham solution or NMDA. Arrowheads indicate GABA A R synaptic clusters. Scale bar, 5 μm. ( f ) NMDA-induced increase of total surface GABA A R average immunoreactivity and GABA A R synaptic cluster integrated fluorescence intensity observed in β3 wt -expressing neurons (black) are prevented by the S383A mutation on β3 subunit (cyan) (total β3 wt : sham=50±5 a.u. per pixel, NMDA=65±2 a.u. per pixel; total β3 S383A : sham=37±2 a.u. per pixel; NMDA=40±2 a.u. per pixel; n =24 in each condition, one-way ANOVA, followed by Newman–Keuls’ post test) (synaptic cluster intensity β3 wt : sham=1,700±190 a.u., NMDA=2,401±131 a.u. ; β3 S383A : sham=1,258±100 a.u. ; NMDA=1,023±96 a.u. ; n =24 in each condition, one-way ANOVA, followed by Newman–Keuls’ post test). ( g ) Comparable trajectories (yellow) of an individual SEP-β3 S383A -containing GABA A R coupled to a QD before and after NMDA treatment. vGAT is represented in red. Scale bar, 1 μm. See also Supplementary Movie 2 . ( h ) Matched MSD over time plot of individual β3 S383A receptors observed at synapses before and after NMDA ( n trajectories =61, 17 neurons, P >0.05, paired t -test). ( i ) Synaptic β3 S383A receptors before and after NMDA treatment exhibit comparable median diffusion coefficient (and IQR) ( n trajectories : before=272; NMDA=263, 17 neurons; P >0.05, Mann–Whitney U -test) and immobile fraction ( P >0.05, Student’s t -test). ( j ) Matched diffusion coefficients of individual β3 S383A receptors present at synapses before and after NMDA ( n trajectories =61 out of 236–272; P >0.05, paired Wilcoxon test). Unless otherwise stated, error bars represent s.e.m. * P <0.05; ** P <0.01; ns, nonsignificant. Full size image To assess the functional role of β3-Ser 383 phosphorylation on chem-iLTP, the effects of NMDA stimulation were tested in neurons expressing β3 S383A , a mutation that prevents the phosphorylation by CaMKII on this residue [34] . Experiments were performed on DIV 16–18 hippocampal neurons transfected with β3 S383A or β3 wt at DIV 7. GABAergic synaptic currents recorded from β3 S383A -expressing neurons were not significantly potentiated after NMDA treatment (10.9±14.6%, n =10; P >0.05, one-way ANOVA, followed by Dunnett’s post test) in contrast to those recorded from β3-expressing neurons (44.6±9.2 %, n =10, from three independent neuronal preparations; P <0.01, one-way ANOVA, followed by Dunnett’s post test; Fig. 3c,d ). In parallel, NMDA stimulation on β3 S383A -containing neurons left unchanged the total surface expression and synaptic clustering of GABA A Rs, assessed by live surface α1 subunit immunostaining as compared with control neurons ( n =24 cells in each condition, from three independent neuronal preparations; one-way ANOVA, followed by Newman–Keuls’ post test; Fig. 3e,f ). In control experiments, we found that the transfection of the β3 subunit did not alter surface GABA A R expression and synaptic clustering, as the basal amount of GABA A Rs synaptic clusters immunoprobed for α1 or β3 subunits in β3-expressing neurons was comparable to those in control (enhanced GFP (EGFP) expressing) neurons ( Supplementary Fig. 5 ). SPT experiments revealed that surface GABA A Rs carrying the β3 S383A point mutation were not immobilized at synapses after chemical induction of iLTP ( Fig. 3g and Supplementary Movie 2 ). In contrast to β3 wt receptors ( Fig. 1f–h ), the confinement, diffusion coefficient and immobile fraction of synaptic β3 S383A receptors were unaffected by NMDA treatment ( n trajectories : before=272; NMDA=263 from 17 neurons; matched observations=61; Fig. 3h–j ). These findings indicate that CaMKII phosphorylation at β3 S383 plays a pivotal role in the accumulation and retention of GABA A Rs at synapses during chem-iLTP. Recruitment of extrasynaptic gephyrin to synapse during iLTP We next investigated whether synaptic GABA A R immobilization during chem-iLTP was associated with an increase in the scaffold protein gephyrin. Immunocytochemical experiments revealed that following NMDA stimulation, the fluorescence intensity, density and area of synaptic gephyrin clusters increased as compared with that of controls. These effects were completely abolished by KN-62 (3 μM) ( n cells: sham=22, NMDA=28, NMDA+KN-62=34, from 4 different neuronal preparations; one-way ANOVA, followed by Newman–Keuls’ post test; Fig. 4a,b ), indicating that the accumulation of gephyrin at synapses during potentiation of inhibition is CaMKII dependent. To corroborate this result and to exclude any concern about the specificity of the antibody used [37] , we quantified gephyrin availability during chem-iLTP by immunocytochemistry with an alternative anti-gephyrin antibody ( Supplementary Fig. 6 ) as well as by live fast-confocal imaging of recombinant gephyrin in an antibody-free assay (see below). Notably, the increase in synaptic gephyrin clustering detected with the mAb3B11 antibody after NMDA treatment was similar to that detected with the mAb7a antibody (synaptic cluster integrated intensity: sham=861.0±41.2 a.u., n =53; NMDA=1096.0±45.5 a.u., n =51; P <0.001, Student’s t -test, Supplementary Fig. 6 ). To assess whether the NMDA-induced increase in synaptic gephyrin involved de novo protein synthesis, western blot (WB) assays were conducted on stimulated neurons in the presence or absence of the protein synthesis inhibitor cycloheximide (CHX, 0.5 mg ml −1 ). Quantitative analysis of gephyrin immunoblots revealed that within 20 min after stimulation, de novo synthesis was not significantly contributing to gephyrin increase (gephyrin intensity: ctrl=100%; NMDA=98.4±14.0%; NMDA+CHX=99.5±18.4%; n =10; P =0.99, one-way ANOVA test followed by Dunn’s post test; Fig. 4c ), whereas at 45 min the total gephyrin protein levels were significantly upregulated as compared with control (gephyrin intensity: ctrl=100%; NMDA=118.4±9.9%; NMDA+CHX=102.5±8.6%; n =10; P =0.04, one-way ANOVA followed by Dunn’s post test; Fig. 4d ). 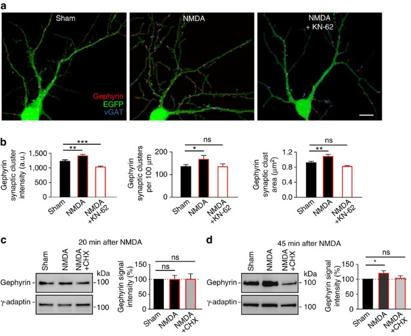Figure 4: During chem-iLTP gephyrin is accumulated at inhibitory synapses. (a) Representative confocal images of hippocampal neurons immunoprobed for gephyrin (red), vGAT (blue) in EGFP-expressing neurons (green). Neurons treated with a sham solution (left), NMDA (middle) or NMDA+KN-62 (right) are compared. Scale bar, 10 μm. (b) Quantification of synaptic gephyrin integrated intensity, cluster density and cluster area in the indicated conditions (n: sham =22, NMDA=28, NMDA+KN-62=34; one-way ANOVA, followed by Newman–Keuls’ post test). (c) Left: representative immunoblotting of total protein levels of gephyrin 20 min after incubation with sham solution or NMDA, in control conditions and on application of CHX to inhibit protein synthesis. Right: quantification of gephyrin protein levels 20 min after NMDA stimulation normalized to sham treatment shows no significant gephyrin upregulation after 20 min (n=10; one-way ANOVA followed by Dunn’s post test,P=0.99). (d) Left: example immunoblotting of total gephyrin levels performed on neuronal lysates 45 min after sham or NMDA stimulation in control conditions and in the presence of CHX. Right: quantification of WB assays described on the left indicates that 45 min after NMDA application gephyrin protein levels are significantly increased (n=10; one-way ANOVA followed by Dunn’s post test,P=0.04). γ-Adaptin immunoreactivity is reported incanddto check equal loading. Error bars represent s.e.m. *P<0.05; **P<0.01; ***P<0.001 and ns, nonsignificant. Figure 4: During chem-iLTP gephyrin is accumulated at inhibitory synapses. ( a ) Representative confocal images of hippocampal neurons immunoprobed for gephyrin (red), vGAT (blue) in EGFP-expressing neurons (green). Neurons treated with a sham solution (left), NMDA (middle) or NMDA+KN-62 (right) are compared. Scale bar, 10 μm. ( b ) Quantification of synaptic gephyrin integrated intensity, cluster density and cluster area in the indicated conditions ( n : sham =22, NMDA=28, NMDA+KN-62=34; one-way ANOVA, followed by Newman–Keuls’ post test). ( c ) Left: representative immunoblotting of total protein levels of gephyrin 20 min after incubation with sham solution or NMDA, in control conditions and on application of CHX to inhibit protein synthesis. Right: quantification of gephyrin protein levels 20 min after NMDA stimulation normalized to sham treatment shows no significant gephyrin upregulation after 20 min ( n =10; one-way ANOVA followed by Dunn’s post test, P =0.99). ( d ) Left: example immunoblotting of total gephyrin levels performed on neuronal lysates 45 min after sham or NMDA stimulation in control conditions and in the presence of CHX. Right: quantification of WB assays described on the left indicates that 45 min after NMDA application gephyrin protein levels are significantly increased ( n =10; one-way ANOVA followed by Dunn’s post test, P =0.04). γ-Adaptin immunoreactivity is reported in c and d to check equal loading. Error bars represent s.e.m. * P <0.05; ** P <0.01; *** P <0.001 and ns, nonsignificant. Full size image Having excluded de novo gephyrin protein synthesis in the first 20 min after NMDA stimulation, the source of gephyrin synaptic increase in the early phase of chem-iLTP expression remains to be assessed. To this purpose, the distribution of mRFP-tagged gephyrin was studied over time before and after NMDA stimulation by live fast-confocal microscopy (see Methods). Hippocampal neurons were transfected with mRFP-gephyrin at DIV 7 and observed at DIV 16–18 after live labelling with an anti-vGAT Oyster650 antibody to visualize presynaptic terminals ( Fig. 5a ). Fluorescence images were acquired every 60 s for 6 min before and for 26 min after NMDA stimulation (see Methods). Data were corrected for fluorescence photobleaching estimated in control experiments by replacing NMDA with a sham solution (11 neurons from 4 independent neuronal preparations). In line with the immunocytochemistry results, we first observed that the fluorescence intensity of mRFP-gephyrin synaptic clusters (exhibiting a juxtaposed vGAT puncta) significantly increased over time after NMDA stimulation ( Fig. 5b,e , see also Fig. 6 and text below). Next, to explore the possibility of gephyrin redistributions during chem-iLTP, mRFP-gephyrin fluorescence at soma and dendrites was quantified over time. We found that the average fluorescence intensity of mRFP-gephyrin in these compartments was not affected by NMDA stimulation (normalized gephyrin fluorescence after/before: soma=1.00±0.03; dendrites: 1.00±0.01, n =13 neurons; P =0.30, Mann–Whitney U -test; Fig. 5c ), thus excluding gephyrin rearrangements between somatic and dendritic areas during chem-iLTP. We next focused on extrasynaptic gephyrin dynamics during chem-iLTP, by quantifying the mRFP-gephyrin fluorescence detected in dendritic areas excluding synaptic clusters. This analysis revealed that NMDA treatment induced a progressive decrease of extrasynaptic gephyrin fluorescence ( Fig. 5d ). Interestingly, this decrease of extrasynaptic gephyrin (computed as the cumulative fluorescence intensity over the dendrite, Fig. 5f ) was on par with the gephyrin intensity increase observed at synapses during chem-iLTP ( Fig. 5g ). Even more importantly, the significant decrease of the extrasynaptic gephyrin fluorescence induced by NMDA stimulation (13 neurons from 4 independent preparations, one-way ANOVA test followed by Dunn’s post test, P =0.006) was paralleled by unaffected total dendritic fluorescence intensity (one-way ANOVA test followed by Dunn’s post test, P =0.36; Fig. 5h ). Altogether, these pieces of evidence indicate that during chem-iLTP, gephyrin is first redistributed from extrasynaptic to synaptic compartments and, on a longer time scale, it is also upregulated. 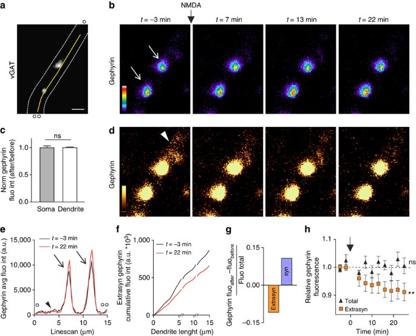Figure 5: Gephyrin redistribution to synapses during chem-iLTP. (a) Example image of presynaptic terminal live staining (with vGAT-Oyster 550) for the localization of inhibitory synapses. Dotted lines depict the profile of the dendrite. The yellow line indicates the position of the linescan reported ine, beginning at (o) and ending at (oo). Scale bar, 2 μm. (b) Pseudocolour images of mRFP-gephyrin fluorescence in the same dendrite as in a at different time points before and after NMDA stimulation (plain arrow). Arrows indicate gephyrin synaptic clusters that increase during chem-iLTP. (c) Normalized gephyrin average fluorescence (after NMDA/before NMDA) observed at soma and dendrites (n=13 neurons;P=0.30, Mann–WhitneyU-test). (d) Gold pseudocolour representation of the same images shown inbwith a different scale to highlight the decrease of extrasynaptic gephyrin (arrowhead) over time. Note that with such scale, synaptic gephyrin clusters are saturated. The arrowhead indicates extrasynaptic gephyrin. (e) Linescans (15 pixels scan width) of gephyrin fluorescence before and 22 min after NMDA stimulation along the line reported ina. The beginning (o) and the end (oo) of the linescans correspond to those ina. The arrows indicate gephyrin synaptic clusters as inb; the arrowhead indicates extrasynaptic gephyrin as ind. (f) Cumulative fluorescence intensity of extrasynaptic gephyrin in the portion of dendrite shown ind. Axis breaks indicate the exclusion of synaptic clusters. (g) NMDA-induced changes in gephyrin intensity shown in b and d at extrasynaptic (extrasyn) compartments are on par with those at synapses (syn). The bar plot represents the difference in normalized gephyrin fluorescence att=22 min andt=−3 min. (h) Quantification of normalized total and extrasynaptic gephyrin fluorescence intensity over time after NMDA application (plain arrow) in 13 neurons (total:P=0.36; extrasynaptic:P=0.006; one-way ANOVA followed by Dunn’s post test for each plot). In live fast-confocal microscopy experiments, photobleach over time was quantified in sham-treated controls (n=11 neurons) and corrected accordingly. Data are expressed as mean±s.e.m. **P<0.01; and ns, nonsignificant. Figure 5: Gephyrin redistribution to synapses during chem-iLTP. ( a ) Example image of presynaptic terminal live staining (with vGAT-Oyster 550) for the localization of inhibitory synapses. Dotted lines depict the profile of the dendrite. The yellow line indicates the position of the linescan reported in e , beginning at (o) and ending at (oo). Scale bar, 2 μm. ( b ) Pseudocolour images of mRFP-gephyrin fluorescence in the same dendrite as in a at different time points before and after NMDA stimulation (plain arrow). Arrows indicate gephyrin synaptic clusters that increase during chem-iLTP. ( c ) Normalized gephyrin average fluorescence (after NMDA/before NMDA) observed at soma and dendrites ( n =13 neurons; P =0.30, Mann–Whitney U -test). ( d ) Gold pseudocolour representation of the same images shown in b with a different scale to highlight the decrease of extrasynaptic gephyrin (arrowhead) over time. Note that with such scale, synaptic gephyrin clusters are saturated. The arrowhead indicates extrasynaptic gephyrin. ( e ) Linescans (15 pixels scan width) of gephyrin fluorescence before and 22 min after NMDA stimulation along the line reported in a . The beginning (o) and the end (oo) of the linescans correspond to those in a . The arrows indicate gephyrin synaptic clusters as in b ; the arrowhead indicates extrasynaptic gephyrin as in d . ( f ) Cumulative fluorescence intensity of extrasynaptic gephyrin in the portion of dendrite shown in d . Axis breaks indicate the exclusion of synaptic clusters. ( g ) NMDA-induced changes in gephyrin intensity shown in b and d at extrasynaptic (extrasyn) compartments are on par with those at synapses (syn). The bar plot represents the difference in normalized gephyrin fluorescence at t =22 min and t =−3 min. ( h ) Quantification of normalized total and extrasynaptic gephyrin fluorescence intensity over time after NMDA application (plain arrow) in 13 neurons (total: P =0.36; extrasynaptic: P =0.006; one-way ANOVA followed by Dunn’s post test for each plot). In live fast-confocal microscopy experiments, photobleach over time was quantified in sham-treated controls ( n =11 neurons) and corrected accordingly. Data are expressed as mean±s.e.m. ** P <0.01; and ns, nonsignificant. 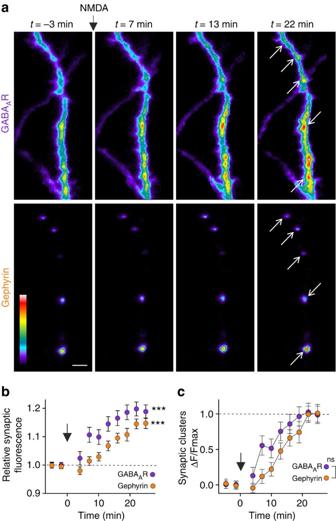Figure 6: Time course of GABAAR and gephyrin synaptic increase during chem-iLTP. (a) Example pseudocolour images of simultaneous live fast-confocal imaging of GABAAR (SEP-β3) and gephyrin-mRFP at different time points in neurons stimulated with NMDA (black arrow). White arrows indicate synaptic clusters. Scale bar, 2.5 μm. Note that, similar toFig. 5b,d, the pseudocolour scale required to see changes in gephyrin cluster intensity does not allow visualization of extrasynaptic gephyrin. (b) Relative GABAAR and gephyrin fluorescence increase over time during chem-iLTP (n=144 areas/time point in 13 different neurons; one-way ANOVA followed by Dunn’s post test,P<0.001 for each curve). The time points include those indicated ina. (c) ΔF/Fmaxplot over time of GABAAR and gephyrin fluorescence intensities shows that increase of GABAAR slightly, although not significantly, precedes that of gephyrin (n=144 areas/time point; synapses; two-way ANOVA followed by Bonferroni post test). In the live fast-confocal imaging experiments, photobleach over time was quantified in sham-treated controls and corrected accordingly. Data are presented as mean±s.e.m. ***P<0.001 and ns, nonsignificant. Full size image Figure 6: Time course of GABA A R and gephyrin synaptic increase during chem-iLTP. ( a ) Example pseudocolour images of simultaneous live fast-confocal imaging of GABA A R (SEP-β3) and gephyrin-mRFP at different time points in neurons stimulated with NMDA (black arrow). White arrows indicate synaptic clusters. Scale bar, 2.5 μm. Note that, similar to Fig. 5b,d , the pseudocolour scale required to see changes in gephyrin cluster intensity does not allow visualization of extrasynaptic gephyrin. ( b ) Relative GABA A R and gephyrin fluorescence increase over time during chem-iLTP ( n =144 areas/time point in 13 different neurons; one-way ANOVA followed by Dunn’s post test, P <0.001 for each curve). The time points include those indicated in a . ( c ) Δ F / F max plot over time of GABA A R and gephyrin fluorescence intensities shows that increase of GABA A R slightly, although not significantly, precedes that of gephyrin ( n =144 areas/time point; synapses; two-way ANOVA followed by Bonferroni post test). In the live fast-confocal imaging experiments, photobleach over time was quantified in sham-treated controls and corrected accordingly. Data are presented as mean±s.e.m. *** P <0.001 and ns, nonsignificant. Full size image Gephyrin synaptic increase requires phosphorylated β3 S383 To investigate the relative timing of NMDA-induced accumulation of GABA A R and gephyrin at synapses, we simultaneously monitored SEP-β3-GABA A R and mRFP-gephyrin synaptic fluorescence over time before and after iLTP induction ( Fig. 6a ) by using the live fast-confocal microscopy approach described above (see also Methods). On NMDA application, the fluorescence of SEP-β3 synaptic clusters increased over time ( n =144 areas/time point in 13 different neurons from 4 independent neuronal preparations; one-way ANOVA test followed by Dunn’s post test, P <0.001; Fig. 6a,b ) and was paralleled by a similar increase of mRFP-gephyrin synaptic cluster intensity ( n =144 areas/time point in 13 different neurons from 4 independent neuronal preparations; one-way ANOVA test followed by Dunn’s post test, P <0.001; Fig. 6a,b ). Data were corrected for fluorescence photobleaching estimated in control experiments by replacing NMDA with a sham solution ( n =120 areas/time point in 11 different neurons from 4 independent neuronal preparations). It is worth pointing out that the results of this antibody-free assay are consistent with those obtained by immunocytochemistry (see also Fig. 1c,d , Fig. 4a,b and Supplementary Fig. 6 ). Next, we calculated the normalized time course of live GABA A R and gephyrin fluorescence increase (ΔF/Fmax) during chem-iLTP ( Fig. 6c , n =144, 13 different neurons from 4 independent neuronal preparations). Unexpectedly, we found that gephyrin increase did not significantly precede GABA A Rs accumulation at synapses ( P =0.49, two-way ANOVA test followed by Bonferroni post test), thus challenging the consolidated idea that adjustments in scaffold availability precede changes in receptor number at synapses. To clarify the functional link between CaMKII activity on β3 subunit and the concerted increase of GABA A R/gephyrin at synapses, we next studied the role of β3 S383 phosphorylation in the accumulation of synaptic gephyrin during chem-iLTP ( Fig. 7a,b ). In β3 S383A -expressing neurons (transfected at DIV 7 observed at DIV 16–18), NMDA did not increase synaptic gephyrin as compared with sham treatment. On the contrary, same protocol applied to neurons transfected with β3 wt induced a significant enhancement of synaptic gephyrin accumulation ( n =24 cells in each condition; one-way ANOVA, followed by Newman–Keuls’ post test; Fig. 7c ). Moreover, the increase in synaptic gephyrin induced by NMDA in β3 wt -transfected neurons was comparable to that in EGFP-transfected neurons (see Fig. 4a,b ), indicating that receptor overexpression does not alter gephyrin synaptic abundance under basal conditions and during chem-iLTP. In control experiments under basal conditions, gephyrin immunoreactivity levels were not affected by β3 overexpression, being indistinguishable among β3 wt -, β3 S383A - and control EGFP-transfected neurons ( Supplementary Fig. 7 ). These data suggest that CaMKII phosphorylation of β3 S383 residue is essential to promote gephyrin accumulation at GABAergic synapses. 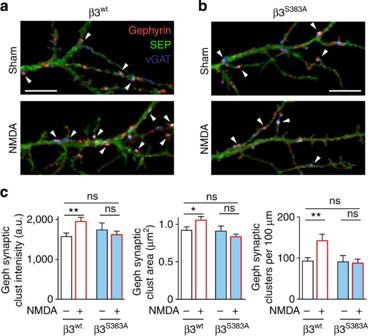Figure 7: Selective CaMKII-dependent phosphorylation of GABAAR β3S383is an essential prerequisite for gephyrin accumulation at synapses during chem-iLTP. (a,b) Representative confocal images of gephyrin (red) and vGAT (blue) immunoreactivity after sham or NMDA treatment in control neurons expressing SEP-β3wt(a) and in neurons expressing SEP-β3S383A(b). Arrowheads indicate synaptic gephyrin clusters. Scale bars, 10 μm (a,b). (c) Quantification of gephyrin immunoreactivity in β3wt- (white) and β3S383A- (cyan) expressing neurons after NMDA treatment as compared with control. Error bars represent s.e.m. (n=24 cells per condition; one-way ANOVA, followed by Newman–Keuls’ post-test) *P<0.05; **P<0.01 and ns, nonsignificant. Figure 7: Selective CaMKII-dependent phosphorylation of GABA A R β3 S383 is an essential prerequisite for gephyrin accumulation at synapses during chem-iLTP. ( a , b ) Representative confocal images of gephyrin (red) and vGAT (blue) immunoreactivity after sham or NMDA treatment in control neurons expressing SEP-β3 wt ( a ) and in neurons expressing SEP-β3 S383A ( b ). Arrowheads indicate synaptic gephyrin clusters. Scale bars, 10 μm ( a , b ). ( c ) Quantification of gephyrin immunoreactivity in β3 wt - (white) and β3 S383A - (cyan) expressing neurons after NMDA treatment as compared with control. Error bars represent s.e.m. ( n =24 cells per condition; one-way ANOVA, followed by Newman–Keuls’ post-test) * P <0.05; ** P <0.01 and ns, nonsignificant. Full size image Gephyrin availability is essential for iLTP Although the phosphorylation of GABA A R-β3 S383 induces gephyrin accumulation at synapses, it remains to be established whether the synaptic increase of gephyrin is necessary for chem-iLTP. To explore the involvement of synaptic gephyrin in chem-iLTP expression, NMDA stimulation was applied to neurons transfected at DIV 7 with a dominant-negative (DN) gephyrin polypeptide, gephyrin 2-188, that hampers gephyrin assembly [38] . In a first set of experiments, we assessed the efficiency of this DN in disrupting endogenous gephyrin clustering ( Fig. 8a ). Gephyrin 2-188 overexpression markedly reduced the density of gephyrin synaptic clusters (ctrl: 112.8±9.6 clusters per 100 μm, n =35; DN: 50.0±6.3 clusters per 100 μm, n =23; P <0.001, Student’s t -test) and also decreased the integrated fluorescence intensity (ctrl: 991.1±36.9 a.u., DN: 820.8±42.8 a.u. ; P =0.005, Student’s t -test) and the area (ctrl: 0.97±0.03 a.u., DN: 0.85±0.03 a.u. ; P =0.005, Student’s t -test) of gephyrin synaptic clusters ( Fig. 8b ). It is worth mentioning that the anti-gephyrin antibody mAb7a, raised using the amino terminus portion of gephyrin did not recognize the gephyrin 2-188 polypeptide in immunocytochemistry. Overexpression of the DN gephyrin 2-188 also affected spontaneous GABAergic synaptic transmission as compared with control. Indeed, in gephyrin 2-188-expressing neurons the amplitude of sIPSCs as well as the frequency was significantly reduced ( n =11 cells in each condition, Student’s t -test; Fig. 8c ). Nonetheless, the peak amplitude and frequency of miniature GABAergic currents recorded in neurons expressing gephyrin 2-188 did not differ with respect to control neurons ( Supplementary Fig. 8 ). Consistent with these observations, gephyrin 2-188 moderately affected the surface expression of GABA A Rs. Indeed, in gephyrin 2-188-expressing neurons the total surface receptor average immunoreactivity (ctrl: 26.4±2.3 a.u. per pixel, n =24; DN: 25.0±1.4 a.u. per pixel, n =24; P >0.05, Student’s t -test) and synaptic cluster density of α1 subunit (ctrl: 42.8±5.0 clusters per 100 μm, n =24; DN: 32.4±5.8 clusters per 100 μm, n =24; 0.05, Student’s t -test; Fig. 8d,e ) were comparable to control neurons, although the integrated intensity of GABA A R synaptic clusters was significantly reduced (ctrl: 1875±151 a.u., n =24; DN: 1609±154 a.u., n =24, P =0.04, Student’s t -test; Fig. 8d,e ). However, disruption of endogenous gephyrin assembly markedly increased the overall GABA A R mobility with respect to control ( Fig. 8f ). In particular, gephyrin 2-188 increased the median diffusion coefficient of total synaptic GABA A Rs (ctrl: 0.022 μm 2 s −1 , IQR=0.004–0.059, n =186 from 12 neurons; geph2-188: 0.040 μm 2 s −1 , IQR=0.016–0.089, n =121 from 10 neurons from 6 independent hippocampal cultures; P =0.005, Mann–Whitney U -test; Fig. 8g ) and reduced the fraction of immobile receptors at synapses (ctrl: 0.31±0.04, n trajectories =186; DN: 0.19±0.02, n trajectories =121; P <0.005, Student’s t -test; Fig. 8g ). Interestingly, the diffusion coefficient of mobile receptors was similar in control and gephyrin 2-188-expressing neurons (ctrl: 0.049 μm 2 s −1 , IQR=0.022–0.099, n =128; DN: 0.050 μm 2 s −1 , IQR=0.024–0.010, n =98; P >0.05, Mann–Whitney U -test; Fig. 8h ), indicating that the main effect of gephyrin impairment on GABA A R mobility is to reduce the trapping of GABA A R at synapses, rather than to change the intrinsic diffusion properties of GABA A Rs. 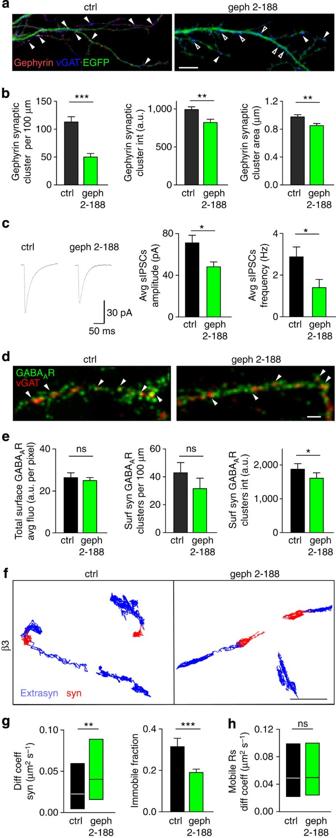Figure 8: Impaired gephyrin clustering affects GABAAR mobility. (a) Representative confocal images of a control neuron expressing EGFP (green, left) and gephyrin 2-188-EGFP (DN) (green, right) immunoprobed for gephyrin (red) and vGAT (blue). Scale bar, 10 μm. Plain arrowheads indicate gephyrin synaptic clusters; empty arrowheads show vGAT puncta lacking juxtaposed gephyrin. (b) Quantification of the immunocytochemical assays comparing gephyrin synaptic cluster density (left), synaptic cluster integrated intensity (middle) and synaptic cluster area (right) in gephyrin 2-188-expressing neurons (n=23) and in control neurons (n=35, Student’st-test). (c) Left: representative traces of sIPSCs recorded from control and gephyrin 2-188-expressing neurons in basal conditions. Right: bar plots of average sIPSCs amplitude and frequency in control (n=11) and 2-188-expressing neurons (n=11), Student’st-test. (d) Representative confocal images of neurons immunoprobed for GABAAR (α1-subunit, green) and for vGAT (red) under control conditions and on impairment of gephyrin assembly. Arrowheads indicate synaptic GABAAR clusters, Scale bar, 1 μm. (e) Quantification of total surface GABAAR average immunoreactivity (left), synaptic cluster density (middle) and integrated intensity of synaptic clusters (right) on gephyrin 2-188 overexpression. (n=24 cells in each condition from three independent hippocampal cultures, Student’st-test). (f) Reconstructed trajectories of β3-containing receptors diffusing at synaptic (red) and extrasynaptic (blue) compartments in control neurons (left) and on gephyrin impairment (right). Scale bar, 1 μm. (g) Median diffusion coefficient (and IQR) of synaptic GABAAR in control (ntrajectories=186 from 12 neurons) and in gephyrin 2-188-expressing neurons (ntrajectories=121 from 10 neurons,P=0.005, Mann–WhitneyU-test) and the corresponding receptor immobile fraction (P<0.005, Student’st-test). (h) Diffusion coefficient (median±IQR) of the mobile receptor population in control and on gephyrin impairment (P>0.05, Mann–WhitneyU-test). Unless otherwise stated data are expressed as mean and error bars represent s.e.m. *P<0.05; **P<0.01; ***P<0.001; ns, nonsignificant. Figure 8: Impaired gephyrin clustering affects GABA A R mobility. ( a ) Representative confocal images of a control neuron expressing EGFP (green, left) and gephyrin 2-188-EGFP (DN) (green, right) immunoprobed for gephyrin (red) and vGAT (blue). Scale bar, 10 μm. Plain arrowheads indicate gephyrin synaptic clusters; empty arrowheads show vGAT puncta lacking juxtaposed gephyrin. ( b ) Quantification of the immunocytochemical assays comparing gephyrin synaptic cluster density (left), synaptic cluster integrated intensity (middle) and synaptic cluster area (right) in gephyrin 2-188-expressing neurons ( n =23) and in control neurons ( n =35, Student’s t -test). ( c ) Left: representative traces of sIPSCs recorded from control and gephyrin 2-188-expressing neurons in basal conditions. Right: bar plots of average sIPSCs amplitude and frequency in control ( n =11) and 2-188-expressing neurons ( n =11), Student’s t -test. ( d ) Representative confocal images of neurons immunoprobed for GABA A R (α1-subunit, green) and for vGAT (red) under control conditions and on impairment of gephyrin assembly. Arrowheads indicate synaptic GABA A R clusters, Scale bar, 1 μm. ( e ) Quantification of total surface GABA A R average immunoreactivity (left), synaptic cluster density (middle) and integrated intensity of synaptic clusters (right) on gephyrin 2-188 overexpression. ( n =24 cells in each condition from three independent hippocampal cultures, Student’s t -test). ( f ) Reconstructed trajectories of β3-containing receptors diffusing at synaptic (red) and extrasynaptic (blue) compartments in control neurons (left) and on gephyrin impairment (right). Scale bar, 1 μm. ( g ) Median diffusion coefficient (and IQR) of synaptic GABA A R in control ( n trajectories =186 from 12 neurons) and in gephyrin 2-188-expressing neurons ( n trajectories =121 from 10 neurons, P =0.005, Mann–Whitney U -test) and the corresponding receptor immobile fraction ( P <0.005, Student’s t -test). ( h ) Diffusion coefficient (median±IQR) of the mobile receptor population in control and on gephyrin impairment ( P >0.05, Mann–Whitney U -test). Unless otherwise stated data are expressed as mean and error bars represent s.e.m. * P <0.05; ** P <0.01; *** P <0.001; ns, nonsignificant. Full size image In another set of experiments we studied the effect of gephyrin disruption on the expression of chem-iLTP. In gephyrin 2-188-expressing neurons, NMDA treatment did not enhance the amplitude of mIPSCs (−4.5±2.6%, n =12, one-way ANOVA, followed by Dunnett’s post test), whereas in GFP-expressing control neurons it induced iLTP (mIPSCs amplitude potentiation 36.7±14.0%, n =14, one-way ANOVA, followed by Dunnett’s post test, Fig. 9a ), as expected. Consistent with this, live immunolabelling of surface α1 subunits revealed that interfering with gephyrin assembly prevented the accumulation of GABA A Rs at synapses after NMDA treatment (synaptic integrated intensity: sham=1,788±228 a.u., n =21; NMDA=1,860±192 a.u., n =23; P >0.05, Student’s t -test, Fig. 9b ). However, despite gephyrin impairment, an increase in the total GABA A R surface expression was still observed after NMDA application in 2-188-expressing neurons (total average intensity: sham=21.6±1.6 a.u. per pixel, n =21; NMDA=27.3±2.9 a.u. per pixel, n =23; P =0.04, Student’s t -test, Fig. 9b ), indicating that gephyrin involvement in chem-iLTP is downstream of receptor exocytosis. Consistent with this interpretation, gephyrin impairment completely abolished NMDA-induced GABA A R immobilization, leaving GABA A R mobility similar to that under basal conditions ( Fig. 9c and Supplementary Movie 3 ). Indeed, no reduction was observed in the confinement of synaptic GABA A Rs during matched observations before and after NMDA application in gephyrin 2-188-expressing neurons ( n trajectories =26 out of 100–118 from 8 neurons; P >0.05, paired t -test at the steady state of the MSD curve, Fig. 9d ). Accordingly, the median diffusion coefficient of all synaptic receptors was not affected after NMDA, as compared with before (before: 0.0535 μm 2 s −1 , IQR=0.0301–0.0895, n trajectories =118; after: 0.0513 μm 2 s −1 , IQR=0.0161–0.1168, n trajectories =100 from 8 neurons; P >0.05 Mann–Whitney U -test, Fig. 9e ). In addition, matched tracking of individual synaptic receptors revealed unchanged diffusion coefficient before and after NMDA treatment in gephyrin 2-188-expressing neurons ( n trajectories =26; P >0.05, paired Wilcoxon test, Fig. 9e ). 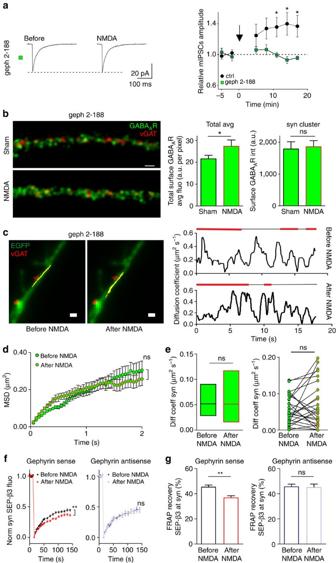Figure 9: Gephyrin impairment prevents chem-iLTP and the associated GABAAR accumulation and immobilization at synapses. (a) Left: representative traces of mIPSCs recorded in a gephyrin 2-188-expressing neuron before and after NMDA. Right: relative amplitude increase of mIPSCs after NMDA application on gephyrin 2-188 (green,n=12) and control (black,n=14) neurons (one-way ANOVA, followed by Dunnett’s post test). (b) Left: representative confocal images of surface GABAAR immunoreactivity (α1-subunit, green) opposed to vGAT (red) in sham and NMDA-treated neurons overexpressing gephyrin 2-188. Scale bar, 10 μm. Right: quantification of the total surface GABAAR average immunoreactivity and synaptic GABAAR cluster intensity in gephyrin 2-188-expressing neurons treated with NMDA or with a sham solution (n=21–23 cells, from three independent neuronal preparations; Student’st-test) (c) Left: representative trajectories (yellow) of an individual GABAAR (β3 subunit-QD) diffusing on a neuron transfected with EGFP-gephyrin 2-188 (green) before and after NMDA application. Presynaptic terminals are represented in red (vGAT). Scale bar, 1 μm. SeeSupplementary Movie 3. Right: diffusion coefficient versus time plots of the GABAAR-QD complex shown on the left before and after NMDA treatment. Lines above the curves represent synaptic (red) and extrasynaptic (black) localization of the particle. (d) MSD versus time plot of matched individual synaptic GABAARs monitored before and after NMDA stimulation in gephyrin 2-188-expressing neurons (ntrajectories=26 from 8 neurons,P>0.05, pairedt-test at steady state). (e) Left: diffusion coefficient (median±IQR) of total synaptic receptors after NMDA treatment (ntrajectories=100) as compared with before (ntrajectories=118, from 8 neurons from 3 independent hippocampal cultures,P>0.05, Mann–WhitneyU-test). Right: matched diffusion coefficients of the same receptors found at synapses before and after NMDA (ntrajectories=26 out of 100–118,P>0.05, paired Wilcoxon test). (f) FRAP over time curves of surface synaptic SEP-β3 receptors before and after NMDA treatment in neurons treated with gephyrin sense (left,n=93–89) and antisense (right) oligonucleotides (left,n=56–55). (g) FRAP recovery before (black) and after (violet) NMDA treatment of synaptic SEP-β3 fluorescence in neurons exposed to the control oligonucleotides (gephyrin sense, left,n=93–89, Student’st-test) or gephyrin antisense oligonucleotides (right,n=56–55, Student’st-test). Unless otherwise stated, data are expressed as means±s.e.m. *P<0.05; **P<0.01; ns, nonsignificant. Figure 9: Gephyrin impairment prevents chem-iLTP and the associated GABA A R accumulation and immobilization at synapses. ( a ) Left: representative traces of mIPSCs recorded in a gephyrin 2-188-expressing neuron before and after NMDA. Right: relative amplitude increase of mIPSCs after NMDA application on gephyrin 2-188 (green, n =12) and control (black, n =14) neurons (one-way ANOVA, followed by Dunnett’s post test). ( b ) Left: representative confocal images of surface GABA A R immunoreactivity (α1-subunit, green) opposed to vGAT (red) in sham and NMDA-treated neurons overexpressing gephyrin 2-188. Scale bar, 10 μm. Right: quantification of the total surface GABA A R average immunoreactivity and synaptic GABA A R cluster intensity in gephyrin 2-188-expressing neurons treated with NMDA or with a sham solution ( n =21–23 cells, from three independent neuronal preparations; Student’s t -test) ( c ) Left: representative trajectories (yellow) of an individual GABA A R (β3 subunit-QD) diffusing on a neuron transfected with EGFP-gephyrin 2-188 (green) before and after NMDA application. Presynaptic terminals are represented in red (vGAT). Scale bar, 1 μm. See Supplementary Movie 3 . Right: diffusion coefficient versus time plots of the GABA A R-QD complex shown on the left before and after NMDA treatment. Lines above the curves represent synaptic (red) and extrasynaptic (black) localization of the particle. ( d ) MSD versus time plot of matched individual synaptic GABA A Rs monitored before and after NMDA stimulation in gephyrin 2-188-expressing neurons ( n trajectories =26 from 8 neurons, P >0.05, paired t -test at steady state). ( e ) Left: diffusion coefficient (median±IQR) of total synaptic receptors after NMDA treatment ( n trajectories =100) as compared with before ( n trajectories =118, from 8 neurons from 3 independent hippocampal cultures, P >0.05, Mann–Whitney U -test). Right: matched diffusion coefficients of the same receptors found at synapses before and after NMDA ( n trajectories =26 out of 100–118, P >0.05, paired Wilcoxon test). ( f ) FRAP over time curves of surface synaptic SEP-β3 receptors before and after NMDA treatment in neurons treated with gephyrin sense (left, n =93–89) and antisense (right) oligonucleotides (left, n =56–55). ( g ) FRAP recovery before (black) and after (violet) NMDA treatment of synaptic SEP-β3 fluorescence in neurons exposed to the control oligonucleotides (gephyrin sense, left, n =93–89, Student’s t -test) or gephyrin antisense oligonucleotides (right, n =56–55, Student’s t -test). Unless otherwise stated, data are expressed as means±s.e.m. * P <0.05; ** P <0.01; ns, nonsignificant. Full size image To confirm these findings, we used chronic administration of gephyrin antisense oligonucleotides (5 μM) from DIV 2 to DIV 16 as an alternative approach to impair gephyrin function [18] , [39] . FRAP experiments performed to assess GABA A R mobility at synapses showed that gephyrin antisense oligonucleotides abolished the NMDA-induced GABA A R immobilization ( Fig. 9f ). Indeed, the SEP-β3 fluorescence recovery observed at synapses in antisense oligonucleotides-treated neurons was similar before and after NMDA treatment (before: 44.7±2.1%, n =56; after: 44.2±2.6, n =55; P >0.05, Student’s t -test). On the contrary, control neurons treated with sense oligonucleotides exhibited reduced FRAP of synaptic SEP-β3 fluorescence after NMDA stimulation (before: 44.5±1.7%, n =93; after: 36.0±1.6%, n =89; P =0.002, Student’s t -test, Fig. 9f,g ). It is worth emphasizing that NMDA-induced GABA A R immobilization observed by FRAP in neurons treated with sense oligonucleotides or transfected with mCherry was similar (compare Fig. 9f,g with Supplementary Fig. 4e,f ). These data reinforce the hypothesis that recruitment of gephyrin to synapses and the consequent accumulation and immobilization of GABA A Rs at synapses are crucial for chem-iLTP expression and suggest that the total population of surface GABA A Rs is involved. Gephyrin and GABA A Rs are upregulated during iLTP in vivo To test the physiological relevance of our observations, we focused on monocular deprivation (MD), a classical in vivo protocol of experience-dependent plasticity. By degrading the spatial vision through the closed eye, brief MD causes loss of responsiveness in principal neurons in the primary visual cortex (V1) accompanied by the potentiation of inhibitory transmission selectively onto pyramidal cells [30] , [31] , [32] . In pigmented rats, a brief MD episode (2 days) at the peak of the critical period for ocular dominance plasticity (P22–P24) has been reported to induce iLTP at synapses between inhibitory fast-spiking interneurons and pyramidal cells in the main thalamorecipient lamina of the visual cortex (layer 4) [30] , [31] , [32] . Here we investigated whether such sensory manipulation also upregulates gephyrin and GABA A R clustering in layer 4 pyramidal cells in V1. To this purpose two independent sets of immunohistochemical assays for gephyrin/GABA/DAPI and for GABA A R/vGAT/GABA/DAPI were performed on brain slices from monocularly deprived pigmented rats, along with age-matched controls ( Fig. 10a,b ). We focused on layer 4 binocular visual cortex (V1b), particularly in the somatic area of pyramidal cells, the neuronal compartment where the vast majority of synapses between fast-spiking interneurons and pyramidal cells are located ( Fig. 10c ). Inhibitory neurons were identified by GABA-positive staining ( Fig. 10a and Supplementary Fig. 9 ) and were excluded from further analysis. In a first set of immunohistochemical experiments the total gephyrin fluorescence intensity (see Methods) was quantified in the maximal projection of confocal stacks. We found that MD slices had higher gephyrin average immunoreactivity compared with control (MD: 17.3±0.7 a.u. per pixel, n =16 slices; ctrl: 13.8±1.3 a.u. per pixel, n =12 slices, P =0.02, Student’s t -test; Fig. 10a,d ). This result was confirmed with a more detailed analysis focusing on the three-dimensional reconstruction of the perisomatic region of each GABA-negative principal cell, showing that the integrated fluorescence intensity of somatic gephyrin in MD slices was larger with respect to control slices (ctrl: 123,379±5,059 a.u., n =474 cells; MD: 152,782±5,341 a.u., n =606 cells; P <0.0001, Student’s t -test, Fig. 10d ). In a parallel set of experiments, the expression and synaptic localization of GABA A Rs was studied to assess whether, also in vivo , potentiation of synaptic inhibition is sustained by increased GABA A R synaptic clustering. Confocal images of sagittal brain slices immunoprobed for GABA A R, vGAT, GABA and DAPI ( Fig. 10b and Supplementary Fig. 9 ) showed a significant increase in total GABA A R average immunoreactivity in the visual cortex of MD animals as compared with aged-matched controls (MD: 29.3±1.6 a.u. per pixel, n =15 slices; ctrl: 21.6±1.3 a.u. per pixel, n =15 slices, P =0.001, Student’s t -test; Fig. 10e ). A specific analysis focusing on the perisomatic region of 3D-reconstructed principal (GABA-negative, see Supplementary Fig. 9 ) cells revealed that the integrated fluorescence intensity of GABA A Rs clusters in the somatic area of principal cells in the V1b region was larger in slices from MD rats than in those from controls (ctrl: 369.8±33.8, n =495 cells; MD: 670.9±48.4, n =552 cells, Student’s t -test). Finally, we observed that the manipulation of the sensory environment of the animal associated with iLTP also significantly increased the density of synaptic GABA A Rs clusters, defined as those juxtaposed to vGAT immunoreactivity (ctrl: 0.57±0.08, n =495 cells; MD: 1.34±0.13, n =552 cells, Student’s t -test). Thus, a brief period of MD, that is sufficient to cause iLTP in layer 4 pyramidal neurons in rat V1, likewise leads to perisomatic upregulation of gephyrin and synaptic GABA A Rs. 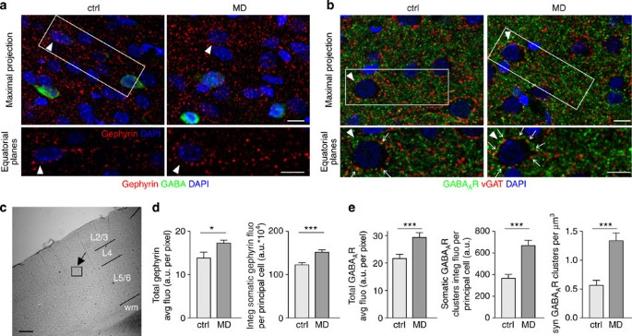Figure 10: Gephyrin and GABAARs are upregulated in the rat visual cortex after brief monocular deprivation (MD). (a,b) Representative confocal images of IHC experiments on slices from control and MD rats immunoprobed for (a): gephyrin (red), GABA (green) and DAPI (blue) or for (b): GABAARs (green), vGAT (red), DAPI (blue) and GABA (seeSupplementary Fig. 9). In both protocols, GABA staining was used to selectively analyse GABA-negativebona fideexcitatory neurons. Top: representative maximal projections of 18 confocalz-stack images (7.5 μm depth) of the binocular visual cortex (V1b) acquired from control and MD samples. Scale bar, 15 μm. Bottom: magnification of the boxes above. Three equatorial planes of the cells indicated by arrowheads are merged. Arrows inbshow GABAAR synaptic clusters. Scale bar, 10 μm in all images. (c) Example of a low magnification (× 4) transmitted light image of the slice used for IHC. The framed box indicates the area acquired at higher magnification (× 60) corresponding to layer 4, V1b. Scale bar, 200 μm. (d) Quantification of gephyrin immunostaining in slices from control (light grey) and MD (dark grey) animals (28 optical planes corresponding to 11.7 μm were considered) (n=12–16, Student’st-test). Total gephyrin average fluorescence (left) and gephyrin-integrated fluorescence detected in the somatic region of each principal cell (right) are shown. (e) Left: total GABAAR average fluorescence intensity in control and MD slices (n=15 in each condition, Student’st-test). Middle: integrated fluorescence intensity of GABAAR clusters identified in the somatic region of principal cells in control and MD slices (n=495 and 552 cells, respectively, Student’st-test). Right: density of synaptic GABAAR clusters in slices from MD rats and age-matched controls (n=495–552 cells, Student’st-test). *P<0.05; ***P<0.001; Student’st-test. Data are expressed as means±s.e.m. Figure 10: Gephyrin and GABA A Rs are upregulated in the rat visual cortex after brief monocular deprivation (MD). ( a , b ) Representative confocal images of IHC experiments on slices from control and MD rats immunoprobed for ( a ): gephyrin (red), GABA (green) and DAPI (blue) or for ( b ): GABA A Rs (green), vGAT (red), DAPI (blue) and GABA (see Supplementary Fig. 9 ). In both protocols, GABA staining was used to selectively analyse GABA-negative bona fide excitatory neurons. Top: representative maximal projections of 18 confocal z -stack images (7.5 μm depth) of the binocular visual cortex (V1b) acquired from control and MD samples. Scale bar, 15 μm. Bottom: magnification of the boxes above. Three equatorial planes of the cells indicated by arrowheads are merged. Arrows in b show GABA A R synaptic clusters. Scale bar, 10 μm in all images. ( c ) Example of a low magnification (× 4) transmitted light image of the slice used for IHC. The framed box indicates the area acquired at higher magnification (× 60) corresponding to layer 4, V1b. Scale bar, 200 μm. ( d ) Quantification of gephyrin immunostaining in slices from control (light grey) and MD (dark grey) animals (28 optical planes corresponding to 11.7 μm were considered) ( n =12–16, Student’s t -test). Total gephyrin average fluorescence (left) and gephyrin-integrated fluorescence detected in the somatic region of each principal cell (right) are shown. ( e ) Left: total GABA A R average fluorescence intensity in control and MD slices ( n =15 in each condition, Student’s t -test). Middle: integrated fluorescence intensity of GABA A R clusters identified in the somatic region of principal cells in control and MD slices ( n =495 and 552 cells, respectively, Student’s t -test). Right: density of synaptic GABA A R clusters in slices from MD rats and age-matched controls ( n =495–552 cells, Student’s t -test). * P <0.05; *** P <0.001; Student’s t -test. Data are expressed as means±s.e.m. Full size image In this study, we addressed for the first time the detailed mechanisms leading to postsynaptic potentiation of GABAergic synapses. Our data highlight an important role for gephyrin and CaMKII activity in iLTP expression. In particular, we show that gephyrin recruitment at synapses is essential for iLTP, but is dependent on CaMKII phosphorylation of the GABA A R β3 S383 residue. As a consequence, GABA A R are accumulated and retained at synapses, thus mediating increased inhibitory synaptic responses. In support of the physiological relevance of the model proposed here, we also report that gephyrin upregulation and increased GABA A R accumulation at synapses are observed in principal cells in the primary visual cortex of rodents after MD, a classical in vivo model of experience-dependent plasticity. These latter results suggest that the molecular mechanisms underlying chem-iLTP in culture also play a role in potentiation of inhibition in vivo . Our finding that during chem-iLTP, gephyrin accumulation at synapses does not precede the increase in synaptic GABA A R number challenges the current view that synaptic receptor accumulation requires pre-available scaffold-docking sites at synapses. This evidence supports a model where GABA A R and gephyrin concomitantly accumulate at synapses during iLTP expression. However, it is not clear whether these two proteins diffuse from the extrasynaptic to the synaptic compartment independently or after formation of GABA A R–gephyrin complexes pre-assembled in the extrasynaptic compartment. This latter possibility has been hypothesized for glycine receptor–gephyrin interactions [40] . The occurrence of GABA A R–gephyrin extrasynaptic complexes could be demonstrated by the ‘parallel’ diffusion behaviour of GABA A R and gephyrin in simultaneous SPT experiments. Unfortunately, as gephyrin is an intracellular protein, these experiments would be technically very challenging. Furthermore, we cannot exclude that technological advances allowing live-imaging experiments with higher temporal resolution than those presented here may unmask a transient temporal mismatch between the relative synaptic accumulation of GABA A Rs and gephyrin. Importantly, we show that the fine tuning of GABA A Rs number at synapses is crucially influenced by gephyrin accumulation during synaptic potentiation, while it is marginally affected by gephyrin availability under basal conditions, at least for the cell type and the GABA A R isoforms we studied. The slight reduction of GABA A R clusters after gephyrin impairment under basal conditions supports the hypothesis that protein(s) other than gephyrin could maintain GABA A R clustering, as previously demonstrated in gephyrin−/− mice [28] , [29] . Accordingly, it has been shown that loss of γ2-containing GABA A Rs led to only a slight reduction of mIPSCs current amplitude [26] . Consistently with this, recent findings emphasized that other proteins, including neuroligin-2, dystrophyin and collybistin, are upstream to gephyrin in the hierarchy of the postsynaptic scaffold protein organization [23] , [25] , [26] , [27] . Under basal conditions, mIPSCs amplitude was not affected after interfering with gephyrin assembly, despite reduced GABA A R cluster intensity and increased GABA A R mobility. This can be explained if unitary presynaptic release does not activate all postsynaptic receptors [41] . As a consequence, a moderate decrease of postsynaptic receptor number would not result in a sizable current amplitude reduction. This hypothesis is substantiated by the fact that sIPSCs, typically evoked by larger GABA release with consequent larger receptor activation, are more sensitive to gephyrin impairment. It is worth mentioning that in our experiments, NMDA could also affect GABAergic currents through the activation of presynaptic NMDARs. Although we cannot directly exclude this possibility, several lines of evidence point in favour of postsynaptic effect of NMDA on GABAergic currents. Indeed, despite the fact that we observed an increase in mIPSCs frequency during chem-iLTP ( Supplementary Fig. 1f ), the persistence of such increase argues against a presynaptic source of this phenomenon [42] . In this concern, it is likely to be that small events previously buried in the noise become sizable after NMDA application and account for the apparent mIPSCs frequency increase. This possibility is also suggested by the fact that NMDA did not affect the frequency of sIPSCs ( Supplementary Fig. 1b ) that show larger signal-to-noise ratio compared with mIPSCs. Finally, the unchanged density of presynaptic inhibitory terminals further supports the lack of significant presynaptic effect following NMDA treatment. The GABAergic system is crucial for neuronal maturation and network formation at early developmental stages [43] . Several lines of evidence indicate that interfering with the early action of depolarizing GABA may lead to alterations of both glutamatergic and GABAergic synapse formation [44] , [45] . Thus, it is possible that the lack of NMDA-induced potentiation of inhibition observed on impairment of endogenous gephyrin could be a consequence of deficits in neuronal development. However, this hypothesis is unlikely in the light of the lack of major changes in the amplitude and frequency of GABAergic synaptic currents under basal conditions on gephyrin impairment. In addition, as gephyrin 2-188 was transfected at 7 days in vitro (DIV), its major protein expression would be expected at DIV8-9, when the GABAergic system is relatively close to mature. This study provides two converging lines of evidence indicating that β3 S383 phosphorylation is a key determinant for chem-iLTP. First, phosphorylation of the β3 subunit residue S383 is enhanced during synaptic potentiation of inhibition. Second, β3 S383A -containing GABA A Rs were not immobilized at synapses after NMDA stimulation and they prevented the recruitment of gephyrin to synapses. These findings show the importance of β3-S383 phosphorylation for the functional interaction of GABA A Rs with gephyrin (and/or with other proteins involved in the synaptic clustering of GABA A Rs) during chem-iLTP and are in accordance with a recent study [36] reporting that overexpression of β3 S383A prevents the potentiation of tonic currents induced by positive allosteric modulation of L-type calcium channels. Importantly, the similarity of the results obtained here with CaMKII inhibition (KN-62, KN-93 and the kinase-dead mutant CaMKII-K42R) and with the non-phosphorylatable β3 S383A -GABA A R suggests that CaMKII phosphorylation of potential substrates other than β3 S383 , such as gephyrin or other scaffold/auxiliary proteins, would not be sufficient for chem-iLTP expression. A study describing that the phosphorylation of Ser270 affects the epitope recognition of the mAb7a antibody [37] raised the possibility that the higher immunoreactivity of synaptic gephyrin after NMDA treatment reported here might reflect an increase in gephyrin phosphorylation, rather than its accumulation at synapses. This possibility is ruled out by the consistency of synaptic gephyrin increase observed during chem-iLTP by immunocytochemistry with an alternative anti-gephyrin antibody (mAb3B11) and by the antibody-free live fast-confocal imaging of recombinant gephyrin. According to our model, during iLTP, CaMKII phosphorylation of β3 S383 promotes the delivery of GABA A Rs to the cell surface, enhances synaptic clustering of GABA A R and favours the assembly of gephyrin clusters at synapses. The documented interaction of gephyrin with several GABA A R subunits, including β3 (refs 21 , 22 , 23 , 24 ) allows speculation that phosphorylated β3 S383 might exhibit enhanced affinity for gephyrin, thus promoting synaptic gephyrin recruitment from extrasynaptic compartments. Additional modulation of receptor-scaffold interactions at synapses during chem-iLTP might involve distinct gephyrin splice variants [46] and changes in synaptic receptor subunit composition [47] as demonstrated for AMPARs [48] . Moreover, the phosphorylation state of gephyrin [37] , [46] , [49] , [50] , [51] due to the activation of different kinases (GSK, CDK5, ERK, Akt2) could further influence synaptic GABA A R mobility by modulating scaffold assembly during chem-iLTP. The evidence that GABA A R β and γ-subunits are directly phosphorylated by CaMKII [3] , [35] , [52] and by other kinases, including PKA, PKC, Src [6] suggests that the phosphorylation of these subunits could add further complexity in receptor–scaffold interactions during iLTP. Importantly, our SPT data demonstrated that in addition to exocytosed receptors, pre-existing surface GABA A Rs are involved in chem-iLTP; after stimulation, these receptors are immobilized at synapses and contribute to increased surface synaptic GABA A R number. This finding represents an important complement to other studies that previously highlighted the role of GABA A R exocytosis in the potentiation of inhibitory transmission [5] , [10] . Assuming that the molecular machinery that brings GABA A Rs to the cell surface is the same under basal conditions and during synaptic plasticity, a phosphoβ3 S383 -dependent modulation of GABA A R intracellular trafficking might be also hypothesized in light of the reduced receptor exocytosis and lack of potentiation in β3 S383A mutants. This would represent an additional mechanism coexisting with the CaMKII phosphorylation-dependent immobilization of pre-existing surface GABA A R identified here. Although the present work and Marsden et al . [5] report that NMDA treatment induces chem-iLTP, NMDAR activation has also been described to be causal for i-LTD [13] , [15] . This differential effect of NMDA on the induction of inhibitory synaptic plasticity can be explained in terms of the degree of NMDAR activation leading to different levels of intracellular Ca 2+ increase. Indeed, moderate Ca 2+ rise induces iLTP [5] , [10] , while higher intracellular Ca 2+ levels (induced by high NMDA concentrations, sustained excitatory activity or high-frequency stimulation) elicit iLTD [13] , [15] , [16] , [53] . In analogy to excitatory synapses [54] , it can be hypothesized that depending on the extent of intracellular Ca 2+ elevation, it is possible to induce either iLTP or iLTD due to differential activation of CaMKII and/or calcineurin, thereby potentiating/inhibiting diverse intracellular pathways [10] . Potentiation of inhibitory synapses correlates with LTD at excitatory synapses triggered by moderate Ca 2+ entry on brief NMDA application [55] . Indeed, similar to previous reports [56] , in our experiments NMDA-treated neurons exhibited significantly reduced spine density compared with sham-treated neurons ( Supplementary Fig. 10 ). Conversely, the same postsynaptic stimulus that induces depression of inhibitory synapses (for example, massive Ca 2+ entry on strong NMDAR activation or high-frequency stimulation) has been reported to concurrently trigger LTP at excitatory synapses [53] , [57] . Concomitant inhibitory potentiation and excitatory depression (or vice versa) in response to the same stimulus suggest that the convergence of signal transduction pathways allows a coordinated control of plasticity at excitatory and inhibitory synapses. Assuming that the Ca 2+ rise responsible for the induction of plasticity of inhibitory synapses occurs through the activation of NMDARs at glutamatergic synapses [2] , the occurrence of either iLTP or iLTD could be influenced by the relative location of excitatory and inhibitory synapses that determines the profile of Ca 2+ concentration sensed by inhibitory synapses. The recent observation that Ca 2+ rise mediated by L-type Ca 2+ channels activates CaMKII and induces potentiation of tonic inhibition [36] raises the intriguing possibility that other events besides NMDAR activation might lead to an adequate intracellular Ca 2+ concentration for iLTP induction. Those events might include back propagation of action potentials [58] and NMDA, Na + , or Ca 2+ dendritic spikes [59] . In addition, it has been recently proposed that the induction of rebound potentiation (RP) obeys to specific temporal patterns of Ca 2+ dynamics [60] . We found that chem-iLTP is associated with GABA A R immobilization at synapses. The functional impact of receptor lateral mobility was first shown by Heine et al . [14] who reported that rapid replacement of desensitized synaptic AMPAR with extrasynaptic receptors by lateral diffusion maintains synaptic responses in face of repetitive synaptic stimulation. This suggests that receptor lateral mobility acts as a frequency-dependent filter of synaptic currents by exerting a stronger reduction of high-frequency synaptic signals with respect to those occurring at lower frequency. As a consequence, the reduction of synaptic GABA A R mobility during iLTP might accelerate the fading of synaptic responses during high-frequency activity by decreasing desensitized receptor replacement at synapses. The evidence that chem-iLTP expression relies on GABA A R recruitment and immobilization at inhibitory synapses reminds of analogous mechanisms occurring at glutamatergic synapses, where LTP is associated with Ca 2+ -dependent immobilization of AMPAR [14] , [17] , likely to be mediated by postsynaptic activation and translocation of CaMKII [61] . Similarly, in the spinal cord, GlyR are immobilized at synapses during potentiation of glycinergic mIPSCs amplitude [62] . However, the same NMDA-based protocol that induces this glycinergic potentiation (which differs from the chemical protocol adopted in this study), fails to potentiate GABAergic transmission and to immobilize GABA A Rs in the spinal cord [62] , whereas it elicits iLTD and dispersal of GABA A Rs from synapses in the hippocampus [13] . As mentioned above, it is likely to be that depending on the level of NMDAR activation (NMDA concentration/exposure time), NMDA can lead to potentiation or inhibition of synaptic currents and modulation of receptor mobility by regulating the concentration profile of intracellular Ca 2+ that may activate different intracellular pathways. Validation of our model of iLTP is provided here by the comparable molecular modifications observed in vitro during NMDA-induced iLTP and those found after in vivo manipulations of the sensory environment known to induce potentiation of inhibition [30] , [31] , [32] . Indeed, the perisomatic upregulation of gephyrin in the principal cells of the rat visual cortex 48 h after brief MD is consistent with the significant increase of gephyrin total protein levels observed 45 min after NMDA treatment in vitro . Similarly, the increased abundance and synaptic clustering of GABA A Rs observed in principal cells in the layer 4 of the binocular visual cortex of MD animals are reminiscent of the increased accumulation of synaptic GABA A Rs in cultured neurons after the chem-iLTP-inducing protocol. Within this framework, an increase in postsynaptic GABA A Rs or gephyrin upregulation have been observed during long-lasting potentiation of somatic inhibition in rat visual cortex during slow-wave sleep [63] and during the extinction of conditioned fear in the basolateral amygdala [64] . The postsynaptic expression of the inhibitory plasticity addressed in the present work can have strong effects at the network level, as iLTP can, in principle, be extended to all inhibitory synapses impinging on the postsynaptic neuron. By clarifying the mechanisms of inhibitory postsynaptic plasticity, this work provides the molecular basis for future studies addressing the role of activity-driven modulation of inhibition in brain microcircuits both under physiological conditions and in neurological disorders such as autism and epilepsy. Animals All experiments were carried out in accordance with the guidelines established by the European Communities Council (Directive 2010/63/EU of 22 September 2010) were permitted by the Italian Ministry of Health and followed the rules approved by the Italian Institute of Technology. All animal surgeries were done in agreement with the Italian Ministry of Health Regulation and Authorization and have been approved by the Italian Institute of Technology. Plasmid constructs SEP-tagged β3 wt was previously described [65] . HA-tagged β3 wt was derived from SEP-tagged constructs by swapping SEP with HA sequence between the NotI and BglII restriction sites at the fourth amino acid of the mature protein. EGFP was expressed from the pEGFP-N1 (Clontech). EGFP-gephyrin 2-188 was obtained as previously described [38] . EGFP-gephyrin and mRFP-gephyrin were kindly provided by Professor E. Cherubini. CaMKII-K42R mCherry was derived from Dr D. Choquet’s gentle gift of CaMKII-K42R-EGFP by swapping EGFP with mCherry between NheI and XhoI restriction sites. β3 S383A was previously described [34] . All constructs were verified by DNA sequencing. Primary neuronal cultures and transfection Cultures of hippocampal neurons were prepared from E18 C57BL/6J mice. Neurons were plated at a density of 45 × 10 3 cells per ml on polylysine pre-coated coverslips and kept in serum-free Neurobasal medium (Invitrogen, Italy) at 37 °C in 7.4 % CO 2 for 16–18 DIV. During this period, half of the medium was exchanged weekly. Neurons were transfected at 7 DIV using Effectene (Qiagen, Germany) following the manufacturer’s protocol. In the experiments involving gephyrin 2-188 overexpression, SEP-tagged β3-subunits were replaced with HA-tagged β3-subunits (HA-β3 wt or HA-β3SA) to be transfected along with EGFP-gephyrin 2-188, to avoid the overlapping fluorescence emission of the EGFP tag and the SEP tag. Gephyrin sense and antisense oligonuclueotides were previously described and characterized [18] , [39] . Antibodies and drugs Anti-GABA A R α1-subunit (directed against an extracellular epitope) from Alomone, Israel (AGA-001) (1:100 for ICC) and from Synaptic Systems, Germany (224 203) (1:2,500 for immunohistochemistry (IHC)); anti-GFP antibody (1:800), anti-MAP2 (1:1,000) and phalloidin-Alexa 546 (1:40) from Molecular Probes, Italy; anti-HA from Roche, Italy (1:50); anti-gephyrin from Synaptic Systems (mAb7a (147,011) (1:150) and mAb3B11 (147,111) (1:1,000) for ICC; mAb7a (147,021) (1:1,000) for IHC) and from BD Bioscience, Germany (clone 45) (1:250 for WB assay); anti-vGAT (1:400 for ICC and 1:1,000 for IHC), anti-vGAT-Oyster550 (1:150), vGAT-Oyster650 (1:150) antibodies were purchased from Synaptic Systems; anti-GABA rabbit (A2052) (1:500) and anti-actin (A2066) (1:40,000) from Sigma, Milan, Italy; anti-GABA guinea pig from Abcam, UK (17,413) (1:1,500); anti γ-adaptin from BD Bioscience (clone 88) (1: 5,000 for WB assay); anti phospho-S383 (1:15,000) and anti β3 (1:15,000) were characterized previously [36] . Fluorescent secondary antibodies (Alexa 488, 568 and 647) against goat, rabbit, mouse and rat IgG, as well as goat F(ab′)2 anti-rabbit IgG conjugate (H+L) highly cross-adsorbed QD655 were from Invitrogen. Horseradish peroxidase-coupled secondary antibodies were purchased from Dianova (1:50,000). BSA, sucrose, HEPES, BAPTA and EGTA were purchased from Sigma. CNQX, Tetrodotoxin (TTX) and KN-62 were purchased from Tocris (Bristol, UK). KN-62 was dissolved in dimethyl sulphoxide to generate a stock solution (30 mM) to be used at a final dilution of 0.01%. Control experiments with vehicle demonstrated that dimethyl sulphoxide at a 0.01% dilution does not affect GABA A R lateral mobility and synaptic accumulation, as well as IPSCs properties. NMDAR stimulation and drug treatments NMDAR activation was used to chemically induce iLTP as previously described [5] . Briefly, stimulation consisted in incubating neurons in a recording solution (see Supplementary Methods ) supplemented with NMDA 20 μM and CNQX 10 μM for 2 min, and allowing 10-, 18- or 43-min recovery in the recording solution. The effects of NMDA stimulation were monitored after the recovery period. When the effects of chem-iLTP induction were tested inICC, NMDA-treated neurons were compared with sham-treated neurons. The electrophysiology data in each experiment were obtained by recording mIPSCs from the same neuron before and after NMDA treatment up to 30 min. In the SPT experiments, two consecutive 1-min-long movies were recorded at each time point ( t −02 and t +18 ) to take into account the variability of the diffusive behaviour of surface receptors. The analysis focused on QD receptor complexes that were present in the visual field before and after NMDA treatment, while those that left or entered the visual field during the 20 min experiments were discarded. An additional analysis focused on matched data obtained from the subset of QD receptor complexes that remained at synapses throughout the experiment duration. This analysis exploited complementary 1-s-long movies (20 frames) acquired every minute during the recovery period, with the specific purpose to univocally identify the same synaptic receptors over time before their final quantification (described above). Inhibition of CaMKII was performed by supplementing the recording solution with KN-62 (3 μM) or with KN-93 (5 μM) for 10 min before NMDA treatment, during NMDA stimulation and during the recovery period. Control experiments with KN-92 (5 μM), the inactive analogue of KN-93, were performed following the same protocol. Electrophysiological recordings Inhibitory miniature and spontaneous postsynaptic currents were recorded in the whole-cell configuration of the patch-clamp technique. External recording solution contained (in mM): 145 NaCl, 2 KCl, 2 CaCl 2 , 2 MgCl 2 , 10 glucose and 10 HEPES, pH 7.4. Patch pipettes, pulled from borosilicate glass capillaries (Hilgenberg, Malsfeld, Germany), had a 4–5 MΩ resistance when filled with intracellular recording solution containig (in mM): 150 KCl, 1 CaCl 2 , 2 MgCl 2 , 1 EGTA, 10 HEPES and 2 Na 2 ATP (300 mOsm and pH 7.2 with KOH). Currents were acquired using Clampex 10.0 software (Molecular Devices, Sunnyvale, CA). sIPSCs and eIPSCs were recorded at room temperature from a holding potential of −60 mV in the presence of CNQX (10 μM) to isolate GABAergic events. mIPSCs were recorded by adding TTX (1 μM) to the same solution used for sIPSCs and eISPCs. Paired patch whole-cell recordings were performed on cultured hippocampal neurons prepared from transgenic mice carrying the tomato dye in PV-positive interneurons. In particular, Parvalbumin-tomato-positive neurons were obtained by breeding Cg-Gt(ROSA)26Sor tm14(CAG-tdTomato)Hze mice (from Jackson Laboratory, USA) carrying a loxP-flanked STOP cassette that prevents the transcription of the downstream red fluorescent protein variant (tdTomato) with 129P2-Pvalb tm1(cre)Arbr mice expressing Cre-recombinase from the endogenous parvalbumin locus (Pvalb). The resulting offspring will have the stop cassette removed in parvalbumin neurons and the consequent expression of tdTomato. eIPSCs were recorded in putative pyramidal neurons following the generation of a single action potential evoked by short (<1 ms) current injection in connected fluorescent PV+ interneurons ( Supplementary Fig1c , left panel). The stability of the patch was checked by repetitively monitoring the input and series resistance during the experiments. Cells exhibiting 10–15% changes were excluded from the analysis. In our electrophysiology recordings, the noise was σ =1.5 pA. Currents were sampled at 20 kHz and digitally filtered at 3 kHz using the 700B Axopatch amplifier (Molecular Devices). mIPSCs and sIPSCs were detected by using the ‘scaled sliding template’ detection algorithm implemented in pClamp10, first descrived by Clements and Bekkers [66] and by setting the ‘detection criterion value’ to 5. Non-stationary fluctuation analysis Peak scaled non-stationary fluctuation analysis (NSFA) was performed on IPSCs recorded in paired patch configuration (see above). Average IPSC was scaled to each eIPSC before computing the variance. The variance around the average was calculated after subtraction of the baseline variance. In these conditions, the parabolic relation between mean and variance is fitted by the function σ 2 =iI−I 2 /N p , where i is the single channel current and N p is the number of open channel [67] . At least 20–30 IPSCs events were used for each experiment. Traces with superimposed spontaneous activity were discarded form analysis. QD labelling QD staining of surface GABA A R was performed according to previously described protocols [17] . Briefly, rabbit anti-GFP or anti-α1 antibody was premixed with anti-rabbit QD 655 (Invitrogen) for 30 min in the presence of caseine (Vectorlab, Italy) to prevent nonspecific binding. The absence of QD labelling when the primary antibody was omitted from ‘QD–antibody premix’ in control experiments indicated that QD binding was ruled by the antibody specificity (data not shown). The specificity of QD labelling was demonstrated by the exclusive binding of anti-GFP-coupled QDs to β3-SEP-transfected neurons, while neighbouring non-transfected neurons were not labelled ( Supplementary Fig. 11 ). Neurons were then incubated with the diluted antibody–QD premix for 2 min at room temperature to obtain a final QD concentration of 0.1 nM. Subsequently, GABAergic synapses were stained by incubating neurons with an anti-vGAT-Oyster550 at 37 °C. Live-cell imaging and QD recording were performed by acquiring 1,200 consecutive frames at 20 Hz with a 512 × 512 pixel EM-CCD camera (9100, Hamamatsu, Japan) using Metamorph software (ver. 7.5, Molecular Devices, USA). The highly diluted QD labelling resulted in <20 QDs per field of view, so that individual QD receptor complexes did not overlap the trajectories of neighbouring complexes. When, occasionally, two QDs were too close to unambiguously reconstruct their individual trajectories, both QDs were discarded from the analysis. During the experiments, neurons were kept at 32 °C in an open chamber and continuously superfused with the recording solution (see below) at 12 ml h −1 . SEP and Oyster550 fluorescence was acquired with 100–200 ms integration time. Samples were illuminated in epifluorescence with a mercury lamp. EGFP, Oyster550 and QD655 fluorescence signals were observed with appropriate excitation (472/30, 543/22 and 435/40 nm, respectively) and emission filters (520/35, 593/40 and 655/15 nm, respectively) (Semrock, Italy) controlled by filter wheels mounted onto an inverted microscope (Eclipse Ti, Nikon, Japan) equipped with a × 60 oil-1.4 numerical aperture (NA) immersion objective. Single-particle tracking For tracking, single QDs, recognized by their diffraction-limited fluorescence spot shape and characteristic blinking, were followed with 50-ms time resolution. QD spatial coordinates were identified in each frame as sets of >4 connected pixels using two-dimensional object wavelet-based localization [68] at sub-diffraction limited resolution (~40 nm) with MIA software based on simulated annealing algorithm [69] . Continuous tracking between blinks was performed with an implemented version of custom software originally written in MATLAB (The Mathworks Inc., Italy) in Dr Choquet’s lab. The method is based on a QD maximal allowable displacement (4 pixels) during a maximal allowable duration of the dark period (25 frames, corresponding to 1.25-s acquisition). This stringent reconnection of trajectories across QD blinking combined with the highly diluted QD labelling have been set to avoid erroneous reconnection of neighbouring QD in the same trajectory and to provide unambiguous observations of individual receptor QD complex trajectories. Receptor trajectories were defined as ‘synaptic’ (or ‘extrasynaptic’) when their spatial coordinates coincided (or not) with those of the localization of the postsynaptic compartment. As inhibitory synapses were identified by presynaptic vGAT live fluorescence labelling (with vGAT-Oyster 550), postsynaptic compartments were defined as a 2-pixel enlargement of vGAT staining. Although the definition of the compartments was diffraction limited, the sub-wavelength resolution of the single particle detection (~40 nm) allowed accurate description of receptor mobility within such small regions. Instantaneous diffusion coefficients, D , were calculated as previously described [70] from linear fits of the n =1–4 values of the MSD versus time plot, according to the equation: MSD (t)=<r2>=4Dt for two-dimensional diffusion. MSD(t) was calculated according to the formula: for reconstructed trajectories of >100 frames using a custom-made software developed by Dr Choquet (Bordeaux, France). To better characterize receptor mobility, receptor QDs have been distinguished into ‘mobile’ and ‘immobile’ populations by using as a threshold the local minimum of the bimodal distribution of synaptic GABA A R diffusion coefficients (0.0075 μm 2 s −1 ) [70] . Next, the diffusive properties of the mobile receptor population were described as their median±IQR, defined as the interval between 25–75% percentile. The immobile receptor population was described by the immobile fraction defined as the relative duration of the residency of a receptor QD in a given compartment with coefficient <0.0075 μm 2 s −1 . ICC and confocal imaging Live staining of surface GABA A R α1, SEP-β3 or HA-β3 subunits was performed by incubating living neurons for 10 min at room temperature with anti-α1, anti-GFP or anti-HA antibodies, respectively, in the recording solution (see below) supplemented with BSA (1%) and sucrose (250 mM) to prevent receptor endocytosis. After fixation with 4% paraformaldehyde (PFA) for 10 min, neurons were incubated with BSA (1%) for 10 min to prevent nonspecific binding followed by an appropriate fluorescence-conjugated secondary antibody for 45 min at room temperature. Control experiments without the primary antibody were performed to test fluorescence signal arising from nonspecific binding of the secondary antibody. Immunostainings of intracellular proteins such as gephyrin (with mAb7a antibody) and vGAT were performed after fixation (PFA 4%), permeabilization (0.2% Triton X-100 for 10 min) and sequential incubation with primary and secondary antibodies. In the immunocytochemical experiments involving the mAb3B11 anti-gephyrin antibody, fixation was performed with PFA 2% for 10 min, followed by conventional permeabilization and immunostaining with the mAb3B11. Subsequently, neurons were fixed again (with PFA 4%) to allow proper vGAT immunostaining. This procedure preserved GFP fluorescence and yielded a gephyrin staining comparable to that obtained with the methanol/acetone fixation suggested by the manufacturer. Secondary antibodies were chosen to minimize fluorophore spectra overlap. Coverslips, mounted in DAKO fluorescent mounting medium, were observed using a Leica TCS SP5 laser scanning confocal microscope with excitation lines from 405-, 488-, 543- and 633-nm lasers (SpectraPhysics) in the sequential mode. Images were acquired using an oil immersion × 63 (NA 1.4) Plan Apochromat objective and analysed using Leica LAS AF software and Metamorph (version 7.5, Molecular Devices). The total average fluorescence intensity of a protein (for example, gephyrin, surface GABA A Rs) in a given neuron was defined as the integrated fluorescence intensity detected in the neuron divided by the neuron pixel area and therefore expressed as au per pixel. Protein clusters (gephyrin and surface GABA A Rs) were defined as synaptic when they exhibited s juxtaposed vGAT puncta within a 2-pixel enlargement. Cluster density represents the number of clusters detected for 100 mm dendrite length. Multicolour live fast-confocal scanning SEP-β3 and mRFP-gephyrin fluorescence signals were simultaneously acquired in an Eclipse Ti microscope (Nikon, Italy) equipped with a × 60 (1.4 NA) and with LiveScan Swept Field Confocal (Nikon, Italy). Samples were illuminated with 488 nm and 568 nm lasers with 500-ms temporal integration. Fluorescence was collected with a 1,004 × 1,002 EM-CCD iXon DU885 (Andor, UK) every 60 s for 6 min before and 26 min after NMDA stimulation. Experiments were conducted at 32 °C. In the quantifications, each data point represents averaged fluorescence of three consecutive images. Synaptic clusters were those exhibiting a juxtaposed live vGAT-Oyster650 signal. Synaptic gephyrin was quantified as the integrated fluorescence intensity of mRFP-gephyrin synaptic clusters. Total mRFP-gephyrin fluorescence was measured in the total area of the neuron. Extrasynaptic gephyrin was measured as the mRFP-gephyrin fluorescence observed in the total neuronal area excluding synaptic clusters. Data were corrected for background noise and for photobleaching over time quantified in control experiments using a sham solution. Monocular deprivation and IHC Pigmented Long Evans rats aged P22 were subjected to MD by means of eyelid suture after avertin anaesthesia (1 ml hg −1 tribromoethanol solution, intraperitoneally). Eyelids were sutured by means of a surgical thread (Ethicon, 6–0) and a topical ointment containing cortisone and antibiotic was applied. Animals were transcardially perfused 48 h after MD using cold (4 °C) 0.1 M PBS followed by 2% PFA solution in the same buffer. Sagittal brain slices from MD and control brains were cut on a freezing microtome at 50 μm thickness. Slices were free-floating immunoprobed for gephyrin and GABA or for GABA A R α1-subunit, vGAT and GABA, and then incubated with appropriate fluorescence-conjugated secondary antibody. Slices were mounted with DAPI-supplemented Vectashield mounting medium and observed by confocal microscopy (see above). When possible, two slices per animal were observed: IHC for gephyrin: n =12 and 16 from 6 and 8 animals in control and MD, respectively; IHC for GABA A R/vGAT: n =15 and 15 from 8 and 8 animals in control and MD, respectively. Images were acquired using a Leica TCS SP5 laser scanning confocal microscope (see above). Initial localization of layer 4 of the binocular part of visual cortex (V1b) was performed with a × 4 objective. Next, one region of interest (ROI) per slice was acquired with an oil immersion × 63 (NA 1.4) Plan Apochromat objective following the confocal microscopy procedure described above. Confocal stacks of 28 optical sections corresponding to 11.7-μm depth ( z resolution 0.42 μm) were analysed using Metamorph (version 7.5, Molecular Devices) and homemade analysis routines running in SigmaPlot 10.0 (Systat Software Inc., UK) and Matlab 7.0 (Mathworks, Italy). GABA staining was used to selectively remove inhibitory GABA-positive neurons from the analysis and to restrict quantification to bona fide excitatory principal cells. Total gephyrin and GABA A R immunoreactivities were quantified as the gephyrin and GABA A R average fluorescence intensities in the maximal projection of 11.7-μm-thick confocal stacks. Integrated somatic gephyrin fluorescence intensity was quantified in the somatic region of each principal cell, indentified in a 6-μm radial enlargement of DAPI staining in each plane. Integrated somatic GABA A R cluster fluorescence intensity refers to the fluorescence intensity of all GABA A R clusters identified in the three-dimensional-reconstructed perisomatic regions of each principal cell. Finally, synaptic GABA A R cluster density represents the number of GABA A R clusters juxtaposed to vGAT immunoreactivity found per μm 3 . The same acquisitions and analysis parameters were applied to all samples. In all quantifications, data were corrected for background. Fluorescence recovery after photobleaching FRAP of SEP-β3 was used to assess the lateral mobility of all surface GABA A R at synapses. To directly demonstrate that in all the experiments conducted at pH 7.4 the use of SEP-β3 allowed the exclusive monitoring of surface GABA A Rs, neurons expressing SEP-β3 were briefly (5 s) exposed to an acidic solution (pH 5.0). The immediate and complete quenching of SEP fluorescence by the acidic solution indicates that surface SEP-β3 receptors were responsible for the fluorescence intensity measured at pH 7.4. Moreover, the sizable increase of SEP-β3 fluorescence observed when neurons were briefly exposed to NH 4 Cl (50 mM) to collapse intracellular pH gradients, confirmed that intracellular SEP-β3 is quenched and does not contribute to the SEP fluorescence during experiments at pH 7.4 ( Supplementary Fig. 4a–d ). Synapses were identified by live staining of vGAT-Oyster 550. Diffraction-limited synaptic regions (juxtaposed to vGAT-Oyster 550 fluorescence) expressing SEP-β3 were photobleached for 5 ms with a 488-nm laser on a Leica TCS SP5 laser scanning confocal microscope equipped with the FRAP module (Leica, Italy). Recovery from photobleaching was monitored by 150 s consecutive acquisitions at 0.5 Hz and normalized to the fluorescence measured before the photobleaching. Residual fluorescence immediately after the photobleaching was set to zero. Recovery curves were corrected for continuous photobleaching and background noise. In each neuron, FRAP was performed on several synapses before and 20 min after NMDA stimulation. Experiments were conducted at 32 °C and at pH 7.4. Acid strip The acid strip procedure, performed on living QD-labelled neurons at the end of the iLTP experiment session (~25 min after QD labelling), consisted in 1 min incubation in pH 2.4 extracellular solution containing 0.5 M NaCl and 0.2 M acetic acid, 10 °C. QDs were imaged (as described above) before and after the acid strip to assess the presence of internalized QD receptor complexes. The efficiency of the acid strip in removing surface antibodies was assessed in control QD-labelled neurons immediately after the labelling (1 min). To verify that internalized receptors could be detected, the acid strip was also performed on neurons kept at 37 °C for 120 min after QD labelling to promote receptor endocytosis. In all conditions, the acid strip was compared with a control treatment consisting in 1 min incubation in cold culture medium. Control treatment did not affect QD labelling. SDS–PAGE and WB assays Cultured hippocampal neurons stimulated with NMDA or with a sham solution were allowed to recover for different durations (10, 18 or 43 min). Samples for GABA A R phosphorylation assays were lysed and harvested in RIPA buffer (50 mM Tris–H–Cl pH 8.0, 150 mM NaCl, 1% Igepal, 0.5% Nadeoxycholate, 0.1 % SDS, 1 mM EDTA) supplemented with protease (P8340- Protease inhibitor cocktail, Sigma) and phosphatase (2 mM Na3VO4, 10 mM NaF) inhibitors. After centrifugation (13,000 r.p.m., 15 min, 4 °C), the protein supernatant was quantified using the micro BCA protein assay kit (Pierce). Total proteins (30 μg) were heated in SDS sample buffer at 50 °C for 10 min and then resolved by SDS–PAGE. Phosphorylated S383 was detected by immunoblotting with rabbit anti phospho-S383 (ref. 36 ), followed by peroxidase-conjugated anti-rabbit IgGs and detection with ECL. Blots were then stripped (Thermo Scientific, PI21059–Restore Western Blot Stripping Buffer) for subsequent probing of total GABA A R β3 (with rabbit anti-β3 IgGs) and actin for equal loading check (with rabbit anti-actin). Incubation with peroxidase-conjugated anti-rabbit IgGs and detection with ECL were repeated to develop total β3 and actin bands. In the experiments aimed at assessing de novo gephyrin protein synthesis, a set of cultured hippocampal neurons were supplemented with 0.5 mg ml −1 cycloheximide (Sigma) during recovery period. All subsequent steps were performed at 4 °C. Cells were rinsed in PBS and harvested in lysis buffer (1 % TritonX-100 (v/v) in PBS supplemented with Complete Mini Protease inhibitor cocktail (Roche)). The supernatant harvested after 30 min centrifugation at 1,000 g was boiled in SDS sample buffer, subjected to SDS–PAGE and analysed by WB assays. The following primary antibodies were used for protein detection: anti-gephyrin and anti-γ-adaptin. Signal intensities were analysed using Image J (version 1.38) analysis software, (National Institutes of Health). Signal intensities were then normalized to the loading control. Statistics Values are given as means±s.e.m. or, in the case of non-normally distributed data, as medians±IQR. Statistical significance was tested using Prism 5.0 Software (GraphPad, USA). Normally distributed data sets were compared using the unpaired two-tailed Student’s t -test, whereas non-Gaussian data sets were tested by two-tailed non-parametric Mann–Whitney U -test. In case of paired non-parametric values, Wilcoxon paired test was used. Statistical significance between more than two normally distributed data sets was tested by one-way ANOVA variance test followed by a Dunnett’s test (to compare data to control) or Newman–Keuls’ test (to compare individual pairs of data) always applying a family-wise 95% confidence interval. In case of paired non-parametric multiple data sets the Kruskal–Wallis test followed by Dunn’s post-hoc test was adopted. Indications of significance correspond to P -values < 0.05 (*), P <0.01 (**), P <0.001 (***) and nonsignificant (ns). For QD tracking, n is the total number of trajectories reconstructed after different experiments performed on multiple neuronal preparations. For ICC, n represents the number of neurons observed. All statistical tests were two-tailed. How to cite this article: Petrini, E.M. et al . Synaptic recruitment of gephyrin regulates surface GABA A receptor dynamics for the expression of inhibitory LTP. Nat. Commun. 5:3921 doi: 10.1038/ncomms4921 (2014).